Human miRNAmiR-675inhibitsDUX4expression and may be exploited as a potential treatment for Facioscapulohumeral muscular dystrophy Facioscapulohumeral muscular dystrophy (FSHD) is a potentially devastating myopathy caused by de-repression of the DUX4 gene in skeletal muscles. Effective therapies will likely involve DUX4 inhibition. RNA interference (RNAi) is one powerful approach to inhibit DUX4 , and we previously described a RNAi gene therapy to achieve DUX4 silencing in FSHD cells and mice using engineered microRNAs. Here we report a strategy to direct RNAi against DUX4 using the natural microRNA miR-675 , which is derived from the lncRNA H19 . Human miR-675 inhibits DUX4 expression and associated outcomes in FSHD cell models. In addition, miR-675 delivery using gene therapy protects muscles from DUX4-associated death in mice. Finally, we show that three known miR-675 -upregulating small molecules inhibit DUX4 and DUX4-activated FSHD biomarkers in FSHD patient-derived myotubes. To our knowledge, this is the first study demonstrating the use of small molecules to suppress a dominant disease gene using an RNAi mechanism. Facioscapulohumeral dystrophy (FSHD) is among the most commonly inherited muscular dystrophies, estimated to affect as many as 870,000 individuals. Classical descriptions of FSHD presentation include progressive muscle weakness in the face, shoulder-girdle and arms, but presentation is often non-uniform [1] , [2] , [3] . For example, 25% develop lower limb or abdominal weakness leading to wheelchair dependence, while others remain ambulant or asymptomatic. Moreover, although FSHD does not typically impact lifespan, some patients may develop life-threatening respiratory muscle complications. Age-at-onset can range from early childhood to adulthood, with earlier onset is often associated with more severe disease [4] . FSHD is caused by aberrant expression of the double homeobox 4 gene ( DUX4 ), which produces a transcription factor that is toxic to skeletal muscle [5] , [6] , [7] , [8] , [9] , [10] , [11] , [12] , [13] . DUX4 is normally functional during the four-cell stage of human development but repressed thereafter in essentially all other tissues, except the testes, skin, and thymus [14] , [15] , [16] , [17] . In skeletal muscles of people with FSHD, genetic and epigenetic factors conspire to permit DUX4 de-repression, which then initiates several aberrant gene expression cascades, including those involved in muscle differentiation and atrophy, oxidative stress, inflammation, and cell death [5] , [6] , [7] , [8] , [9] , [13] , [18] , [19] , [20] , [21] . There are currently no approved treatments that slow FSHD progression or improve muscle weakness. The most direct route to FSHD therapy will involve inhibiting DUX4 in muscle. Gene silencing by RNA interference (RNAi) is one powerful approach to inhibit DUX4 . RNAi is mediated by ~22 nucleotide (nt), non-coding microRNAs in complex with cellular gene silencing machinery, which together are called the RNA-induced silencing complex (RISC). The microRNA component of RISC base-pairs with target transcripts to trigger sequence-specific gene silencing. Importantly, artificial microRNAs can be engineered to trigger RNAi against disease genes. Historically, RNAi-based therapies have relied upon two major strategies to silence dominant disease genes: (i) delivery of siRNA oligonucleotide drugs to permissive target cells or tissues; or (ii) gene therapy in which designed microRNA or shRNA expression cassettes are delivered with viral vectors and expressed intracellularly. To date, three oligonucleotide-based RNAi drugs—Alnylam’s Patisiran, Oxlumo, and Givlaari—are FDA approved, while several promising gene therapy strategies for dominant diseases are still emerging. Using either strategy for FSHD therapy requires delivery of an RNAi product to muscle. Currently, intact muscle is a challenging target for oligonucleotide delivery, but importantly, AAV gene therapy vectors can achieve widespread and long-term transduction of virtually the entire musculature following a single systemic injection. Thus, gene therapy is currently the best approach for delivering an inhibitory RNA to muscle. Nevertheless, the relative permanence of gene therapy could also be a disadvantage; for example, if unwanted side effects developed from inhibitory RNA over-expression, it is currently impossible to turn the vector off or down. Here we pursued an alternative approach to induce RNAi against a dominant disease gene that circumvented delivery problems inherent with oligo-based RNAi systems, and would potentially allow tunability or stoppage of treatment if deleterious effects emerged. Specifically, we hypothesized that the DUX4 transcript may be naturally regulated by one or more of the 1917 known endogenous human microRNA genes, and that it may be possible to upregulate a DUX4 -targeting microRNA with a small molecule, thereby offering a potential drug-based RNAi treatment for FSHD. Unfortunately, prior to this study, no endogenous microRNAs targeting DUX4 had been identified. We, therefore, initiated this study with the goal of identifying endogenous human microRNAs capable of silencing DUX4 . To do this, we used bioinformatics tools to predict prospective DUX4 -targeting human miRNAs and then empirically tested their ability to silence DUX4 . Among numerous candidates tested, we identified miR-675 as a DUX4 regulator. Here, we provide evidence that miR-675 directly targets DUX4 mRNA, inhibits DUX4-responsive biomarkers, and counteracts DUX4-induced toxicity in skeletal muscle and non-muscle cells. In addition, using AAV-based gene therapy, we show that miR-675 can inhibit DUX4-associated histopathology in an FSHD mouse model. Finally, we validated previous studies showing that miR-675 could be increased by estrogen/progesterone and melatonin, and then used these small molecules to upregulate endogenous miR-675 and decrease DUX4 and DUX4-responsive biomarkers in human FSHD myotubes. To our knowledge, this is the first study demonstrating the use of small molecules to suppress a dominant disease gene using RNAi. This study supports translating miR-675 gene and drug therapies as prospective treatments for FSHD, and justifies identifying additional microRNAs that could be exploited for FSHD therapy. Furthermore, this work establishes a potential playbook to develop RNAi-based small molecule therapies for other dominant diseases. MicroRNA screen identifies human miR-675 as a DUX4 inhibitor To investigate the hypothesis that DUX4 was regulated by endogenous miRNAs, we first used the miRNA target prediction algorithm miRBase to identify miRNAs potentially targeting DUX4 3′ end sequences [22] . We tested 23 predicted microRNAs using a dual-luciferase reporter assay, but unfortunately none caused strong DUX4 silencing (details in Supplementary Note 1 and Supplementary Fig. 1 ). We next tested an alternative target prediction algorithm, called PITA ( https://genie.weizmann.ac.il/pubs/mir07/mir07_prediction.html ), which attributes higher rank scores to miRNAs with multiple putative binding sites on a target transcript [23] . We also expanded the sequence search to include the entire DUX4 ORF and 3′UTR, as data emerged suggesting that miRNA regulation can also occur in coding regions [24] . Hsa-miR-675 was among the top hits predicted by PITA, with 14 putative binding sites located throughout the DUX4 ORF and 3’ UTR , including several with potentially high affinity. Based on these data, we focused on miR-675 as our top candidate from the PITA algorithm and switched our Luciferase assay screening strategy to include a construct containing all DUX4 pre-mRNA sequences (ORF and 3’ UTR), including potentially retained introns (called DUX4-FL, where FL = full-length). We then tested the ability of miR-675 to silence DUX4 sequences by luciferase assay in co-transfected HEK293 cells. To deliver miR-675 to cells, we initially used a U6 promoter-driven miR-675 expression plasmid (U6.MIR675), as well as a construct expressing the miR-675 precursor, the lncRNA H19 (CMV.H19) (Fig. 1a ). Importantly, U6.MIR675 and the miR-675 precursor H19 reduced DUX4-FL luciferase activity by 35 ± 3% and 36 ± 2%, respectively ( P < 0.0001, ANOVA, N = 3), while the miLacZ negative control had no impact (Fig. 1a ). As an additional control, we found that U6.MIR675 had no impact on Renilla luciferase that lacked DUX4 sequences, indicating that it does not target Renilla luciferase alone (RenLuc-backbone). The level of knockdown achieved by miR-675 against a DUX4 -attached luciferase target was the best we had so far observed from a natural microRNA, but still did not approach the >80% knockdown elicited by miDUX4.405 , which contains 22 nt of perfect complementary with DUX4 and was designed for optimal gene silencing [21] , [25] , [26] , [27] (Fig. 1b ). Since the PITA algorithm predicted binding sites in both the DUX4 ORF and 3 ′ UTR regions, we also tested U6.MIR675 against the Renilla luciferase constructs containing only the DUX4 ORF (DUX4 ORF) or DUX4 3′UTR (DUX4 3′UTR). U6.MIR675 significantly silenced each construct by 34 ± 2% and 24 ± 5%, respectively ( P < 0.0001, ANOVA, N = 3) (Fig. 1b ). These results supported prior evidence that natural miRNAs can initiate silencing of target genes through base pairing sequences in the ORF as well as the 3 ′ UTR [24] . Finally, there are two species of miR-675 that originate from the H19 precursor, miR-675-5p and miR-675-3p . Only miR-675-5p was predicted to regulate DUX4 and we confirmed these results empirically (Supplementary Note 2 and 3 and Supplementary Fig. 2a, b ). We also tested the functionality of our U6-driven expressing plasmids, by measuring the expression of their known target genes SMAD1 , SMAD5 , and CDC6 [27] (Supplementary Fig. 2c ). Fig. 1: miR-675 targets the DUX4 ORF and 3 ′ UTR . a RenLuc-DUX4-FL dual-luciferase reporter and CMV.H19 constructs, and U6.MIR675, H1.MIR675, U6.MIR675-3p, and U6.MIR675-5p miRNAs. RenLuc-DUX4-FL contains DUX4 ORF and 3 ′ UTR sequences fused to Renilla luciferase after the stop codon. Exons 1–3 are indicated (Ex1,2,3). *SD5 indicates silent mutation of a cryptic splice donor in Renilla luciferase. Firefly luciferase is used as transfection control. b U6.MIR675 reduced relative Renilla luciferase activity in constructs containing full-length DUX4 , DUX4 ORF only, or DUX4 3’ UTR only (35 ± 3%, 34 ± 2%, and 24 ± 5%, respectively; P < 0.0001). H19 reduced relative Renilla luciferase activity from the RenLuc-DUX4-FL by 36 ± 2% ( P < 0.0001). All readings were normalized to Firefly luciferase and then to the milacZ negative control. U6.MIR675 did not reduce relative Renilla luciferase activity from the non-targeting RenLuc control plasmid (RenLuc). The U6.miDUX4.405 positive control is a published artificial microRNA with robust DUX4 silencing activity. Data indicate mean luciferase activity ± SEM ( N = 3 independent experiments). c Relative Renilla luciferase activity was reduced in a dose-dependent manner by two miR-675 constructs: U6.MIR675 and H1.MIR675. Molar ratios of miRNA to reporter plasmid are indicated and data normalized to the miLacZ negative control. U6.MIR675 significantly reduced relative Renilla luciferase activity by 23 ± 3% (10:1 ratio), 29 ± 3% (20:1), and 34 ± 3% (40:1). H1.MIR675 performed better at lower doses, reducing relative Renilla luciferase activity by 42 ± 4%, 39 ± 5%, and 55 ± 3%. All samples were significantly different from the miLacZ control ( P < 0.0001). Data represent mean normalized Renilla luciferase activity ± SEM ( N = 4 independent experiments). d Droplet digital PCR (ddPCR). H1.MIR675 significantly reduced DUX4 mRNA levels by 71 ± 2% ( P < 0.0001, ANOVA, N = 3) compared to the miLacZ negative control, 48 h following transfection of HEK293 cells with a 1:3 ratio of CMV.DUX4-FL/CMV.eGFP and H1.MIR675. Results represent the average absolute DUX4 mRNA concentration (copies/µL) ± 95% poisson confidence interval. Data represent mean relative concentration (copies/μL) ± SEM ( N = 3 independent experiments). For b – d , One-way ANOVA followed by Dunnett’s multiple comparison tests were performed for statistical analyses. e Northern blot using RNA extracted from HEK293 cells transfected with the indicated expression plasmids. U6.miGFP is a negative control. Source data are provided as a Source data file. Full size image To confirm the U6.MIR675 results, we tested a second miR-675 expression construct, utilizing the H1 promoter instead of U6. H1.MIR675 performed consistently better than the original U6.MIR675 construct, reducing relative Renilla luciferase activity by 55 ± 3% (1.6 ± 0.2-fold better than U6.MIR675, P < 0.0001, ANOVA, N = 4) (Fig. 1c ). Using the CMV.DUX4-FL/CMV.eGFP, we also used droplet digital PCR (ddPCR) and QPCR to confirm that miR-675 significantly reduced DUX4 mRNA expression in co-transfected HEK293 cells (Supplementary Note 4 , Supplementary Fig. 9 and Fig. 1d ). To understand the difference in silencing produced by U6.MIR675 and H1.MIR675, we performed small transcript northern blots using RNAs isolated from HEK293s transfected with each construct. The H1.MIR675 construct produced 13-fold and 23-fold more full-length and mature miR-675 compared to U6.MIR675 at 24 h and 48 h post-transfection, respectively (Fig. 1e ). In addition, the mature miR-675 species from both constructs were not identical in size, suggesting differential processing by microRNA biogenesis machinery. The low abundance of mature miR-675-5p from U6.MIR675 could explain the low levels of inhibition when targeting the fully complementary target sequence (miR-675R). (Supplementary Fig. 2d ). Based on these data, H1.MIR675 became our lead expression system for all subsequent experiments. miR-675-5p has multiple binding sites within the DUX4 ORF and 3 ′ UTR The PITA algorithm predicted 14 miR-675 binding sites on DUX4 [23] . We confirmed these predictions with a second platform, RNAHybrid, and then used these data to develop an in vitro binding assay to empirically identify functional miR-675 target sites on DUX4 (Supplementary Data 1 and Supplementary Fig. 3 ) [28] . To do this, we developed a molecular beacon-binding assay in which the miR-675-5p mature sequence was used as a DNA molecular beacon and the predicted target sites were incorporated individually in single stranded oligonucleotides (Fig. 2 ). Mature miR-675 had significant binding affinity ( K d ) with 8 of the 14 predicted DUX4 target sites (Fig. 2 ). Two target sites were located in the 3′UTR (TS1340 and TS1471) and six were in the DUX4 ORF (TS527, TS649, TS668, TS754, TS780, and TS1004). miR-675-5p showed highest binding affinity to TS780 in the DUX4 ORF ( K d = 6 ± 1 µM) and TS1471 in the 3′UTR ( K d = 3 ± 1 µM) (Fig. 2b, c ). Fig. 2: miR-675-5p targets multiple binding sites in the DUX4 ORF and 3 ′ UTR . a Schematic of DUX4 sequence showing predicted target site (TS) positions for miR-675-5p . b (Left) Molecular beacon binding assay used to determine miR-675-5p binding to DUX4 . Unbound, the molecular beacon folds into a stem loop structure that brings the ZenBHQ quencher in close proximity to a the 6FAM fluorophore, thereby preventing 6FAM fluorescence. We incorporated the mature sequence of miR-675-5p in the MB loop sequence. Hybridization of the MB to a complementary DUX4 target sequence separates the fluorophore and quencher, allowing fluorescence emission, which is quantified as a measure of binding. (Right) The graph shows binding of the mature miR-675-5p molecular beacon to target sites shown in ( a ). miR-675-5p bound 8 DUX4 target sites (6 in the ORF and 2 in the 3′UTR). Six predicted TS did not bind to miR-675-5p (Supplementary Fig. 3b and Supplementary Data 1 for TS position and sequence). The TS neg. ctrl is a random sequence. Curves are fit into one site-specific binding with Hill slope equation. Each data point represents mean ± SD ( N = 3 independent experiments). c Base-pairing of miR-675-5p and predicted DUX4 target sites used in the molecular beacon assay. The binding affinity ( K d ) of miR-675-5p molecular beacon to each target site was determined by subtracting background fluorescent signal from the molecular beacon signal (MBS), expressed in relative fluorescent units (RFU). The K d corresponds to the TS concentration (μM) required to reach half of maximum fluorescence. We generated RNA “mimic” bases in the miR-675-5p :TS pair and replaced “G” nucleotides with “A” nucleotides (in gray) whenever the “G” is facing a “T” [29] . Source data are provided as a Source data file. Full size image miR-675 inhibits DUX4 mRNA and protein expression Luciferase reporter and in vitro binding assays suggested that miR-675-5p and the H19 precursor regulated DUX4 expression. In these experiments, DUX4 sequences were present out of context, either attached as the 3’ UTR of Renilla luciferase or embedded within an oligonucleotide. We, therefore, sought to confirm miR-675 -mediated silencing against a wild-type DUX4 target and used western blotting as a secondary gene expression outcome measure. To do this, we co-transfected HEK293 cells, which do not normally express polyadenylated DUX4 , with a DUX4 expression plasmid and various miR-675 expression constructs. To express DUX4 , we constructed a plasmid containing a CMV promoter driving full-length DUX4 fused with a COOH-terminal V5 epitope, and included on the same plasmid a CMV-driven eGFP gene, which was used to normalize transfection efficiency (CMV.DUX4-FL/CMV.eGFP, aka DUX4/eGFP). We then performed a series of unblinded and blinded co-transfections of the DUX4/eGFP plasmid with various miR-675 expression constructs, or controls, into HEK293 cells. Specifically, we transfected 3 different plasmids expressing pri-mir-675 from different promoters (CMV, H1, and U6 promoters); two constructs engineered to preferentially express the −5p or −3p strands of miR-675 (U6.MIR675-5p and U6.MIR675-3p); CMV.H19; the U6.miDUX4.405 artificial microRNA positive control; a U6.miLacZ negative control; and two oligonucleotide miR mimics, which were essentially siRNAs ( miR-675-5p mimic and miR negative control mimic). We then collected protein extracts 48 h later and performed western blotting using antibodies to detect V5 epitope-tagged DUX4 protein (anti-V5) and eGFP. In total, we performed 6 independent transfections, protein collections, and western blot experiments on different days over the course of several weeks. The last four confirmatory experiments were performed using a blinded design, as described in the Methods section. If miR-675 did indeed suppress DUX4 expression, we were expecting mild to modest inhibition, as natural microRNAs typically contain sequence mismatches with target genes and do not direct gene silencing as efficiently as engineered microRNAs containing 22 nt miRNA:mRNA binding sites (e.g., miDUX4.405 ). Indeed, the miDUX4.405 positive control reduced DUX4 protein by 93 ± 4% ( P < 0.0001, ANOVA, N = 6), as we previously described [21] , [29] (Fig. 3a ). Unlike miDUX4.405 , miR-675 did not contain perfect complementarity with DUX4 at any predicted binding site (Fig. 2c ), and so we were surprised to find that the H1.MIR675 expression plasmid produced robust DUX4 gene silencing of 91 ± 4% ( P < 0.0001, ANOVA, N = 6), similar to that of miDUX4.405 (Fig. 3a and Supplementary Fig. 4 – 8 ). All other miR-675 constructs, including H19 and the miR-675-5p mimic, reduced DUX4 protein expression but with variable and more modest efficiencies, ranging between 35 and 53%. As expected, the negative controls, U6.miLacZ and miR negative control mimic, did not inhibit DUX4 protein levels (Fig. 3a and Supplementary Fig. 4 – 8 ). Variability in expression and processing of primary miR-675 transcripts into mature miR-675-5p sequences could account for the differences in silencing capability among the various miR-675 expression constructs (Fig. 1e ). Fig. 3: miR-675-5p specifically targets DUX4 and reduces its protein and mRNA levels in vitro. a , b Blinded western blots detecting V5 epitope-tagged DUX4 and an eGFP transfection control in the presence of miR-675 or control constructs. a Proteins were harvested from HEK293 cells 48 h after co-transfection with the CMV.DUX4-FL/CMV.eGFP expression plasmid and indicated miR-675 or control plasmids. Black boxes, AAV2 inverted terminal repeats (ITR). CMVp, cytomegalovirus promoter. Western blot membranes were stained with antibodies to the V5 epitope tag (to detect DUX4.V5) or eGFP. DUX4 protein was reduced in cells treated with CMV.H19 (35 ± 7%, P = 0.0007, N = 5 independent replicates), miR-675-5p mimic (36 ± 9%, P < 0.0001, N = 3), CMV.MIR675 (53 ± 9%; P < 0.0001, N = 4), U6.MIR675 (49 ± 8%; P < 0.0001, N = 5), and U6.MIR675-5p (42 ± 2%; P = 0.0004, N = 5). H1.MIR675 showed the highest DUX4 inhibition with an average of 91 ± 4% ( P < 0.0001, N = 6), similar to U6.miDUX4.405 (93 ± 4%, P < 0.0001, N = 6). The U6.MIR675-3p construct did not significantly inhibit DUX4 protein levels (11 ± 7%, P = 0.6286, N = 5). b MiR-675 specifically reduced DUX4 expression via target engagement. MiR-675 -resistant DUX4 constructs expressing full-length DUX4 protein or the Renilla luciferase- DUX4 reporter (CMV.DUX4-miR-675Res and RenLuc-DUX4.ORF-miR-675Res) contain silent mutations in miR-675 target site 780 (TS780) and lack miR-675 binding sites in the DUX4 3′UTR. Western blots show that miR-675 expression constructs did not significantly reduce miR-675 -resistant DUX4 ( P = 0.9997), while the U6.miDUX4.405 positive control, which had intact binding sites on DUX4 , reduced mean DUX4 protein levels by 90 ± 6% ( P = 0.0003). Similarly, increasing doses of the H1.MIR675 plasmid did not significantly silence the miR-675 -resistant Renilla luciferase target ( P = 0.3467 for the 14:1 miR-675:DUX4 ORF-miR-675Res ratio). Blots shown represent 6 ( a ) and 3 ( b ) independent blots (additional blots in Supplemental Data ). DUX4 protein (DUX4p) was reported as mean % expression ± SEM and plotted above each representative image. Luciferase assay results ( b ) represent mean relative Renilla luciferase activity ± SEM, normalized to the miLacZ negative control ( N = 3 independent experiments). For a , b one-way ANOVA followed by Dunnett’s multiple comparison tests were performed for statistical analyses. TS780WT: wild-type TS780 sequence. TS780M: TS780 sequence with silent point mutations colored in gray. ΔTS780: deleted TS780. Source data are provided as a Source data file. Full size image To confirm the western blot findings and test the specificity of miR-675 repressive activity on DUX4 , we introduced silent point mutations in the strongest miR-675-5p binding site on DUX4 , target site 780 (TS780) (Fig. 2 and Supplementary Fig. 3b ). These changes were designed to make the mutated TS780 sequence (TS780M) unrecognizable by miR-675-5p . Moreover, in the same construct, the DUX4 3’UTR was omitted, thereby eliminating the other validated high affinity binding site for miR-675 (TS1471) as well as a second binding site with lower affinity (TS1340). We named this construct CMV.DUX4-miR-675Res (where miR-675Res = miR-675 resistant). We cloned a similar construct in which the TS780 was deleted from our DUX4 ORF luciferase reporter plasmid (RenLuc-DUX4 ORF-miR-675Res) (Fig. 3b ). We used the same transfection strategy and outcome measures (western blotting or luciferase assay) described above but replaced the wild-type DUX4 expression plasmids (i.e., DUX4/eGFP and RenLuc-DUX4-FL) with the miR-675 resistant analogs (CMV.DUX4-miR-675Res/CMV.eGFP and RenLuc-DUX4 ORF-miR-675Res). Importantly, as measured by western blot and luciferase assay, none of the miR-675 constructs were capable of suppressing DUX4 protein expression and relative Renilla luciferase activity from the miR-675- resistant mutants (Fig. 3b ). Together, these results confirmed the specificity of miR-675-5p -mediated DUX4 repression. miR-675 and its precursor H19 protected HEK293 from DUX4-induced cell death and inhibited DUX4 transactivation DUX4 encodes a transcription factor that is toxic to numerous cells and tissues from multiple organisms, leading to cell death through apoptosis and possibly other mechanisms [6] , [7] , [9] , [30] , [31] , [32] , [33] , [34] , [35] . Indeed, HEK293 cells are killed by DUX4 over-expression, and since miR-675 can silence DUX4 expression, we hypothesized that it could protect HEK293 cells from DUX4-induced cell death. To investigate this, we co-transfected HEK293 cells with H1.MIR675 and CMV.DUX4 expression plasmids, and measured cell viability over time using a Trypan blue cell viability assay (Fig. 4a ). Cells co-transfected with DUX4 and a negative control showed 23 ± 2% ( P < 0.0001, ANOVA, N = 3) and 58 ± 1% ( P < 0.0001, ANOVA, N = 3) cell death by 48 and 62 h (our longest time point), respectively, when compared to the mock-transfected cells (No DUX4 ). However, H1.MIR675 significantly protected HEK293 cells from DUX4-induced cell death up to 62 h after transfection as only 14 ± 1% of cells were dead ( P < 0.0001, ANOVA, N = 3) similar to our positive control U6.miDUX4.405 that allowed the death of only 13 ± 1% of cells ( P < 0.0001, ANOVA, N = 3). Fig. 4: miR-675 protects cells from DUX4-induced cell death. a Cell viability assay in HEK293 cell transfected with indicated plasmids. Cell death was measured by counting Trypan blue-stained cells over the indicated time course and calculated by subtracting the number of dead cells from the total number of cells plated per well. No significant difference in cell viability was seen before 36 h of transfection. Cells co-transfected with DUX4 and the control pciNeo plasmid showed 23 ± 2% ( P < 0.0001) and 58 ± 1% ( P < 0.0001) cell death by 48 and 62 h, respectively, when compared to the mock-transfected cells (No DUX4 ). However, co-transfection with DUX4 and H1.MIR675 or U6.miDUX4.405 protected HEK293 cells from DUX4-induced cell death, as only 9 ± 2% and 6 ± 2% of cells were dead by 48 h, respectively, and slightly increased by 62 h. These values were not significantly different from mock-transfected HEK293s but represented significant protection from cell death compared to the DUX4 + pciNeo control ( P < 0.0001 for both H1.MIR675 and U6.mi405). Two-way ANOVA followed by Tukey’s multiple comparison tests were performed for statistical analyses. Results were reported as the mean cell viability ratio ± SEM ( N = 3 independent experiment). b Caspase-3/7 assay 48 hrs after co-transfection of HEK293 cells with DUX4 expression plasmid and either U6.miLacZ, U6.miDUX4.405, H1.MIR675, or CMV.H19. The U6.miLacZ negative control failed to protect cells from Caspase-3/7 activation (2.2 ± 0.1-fold increase; P < 0.0001) compared to mock-transfected cells. In contrast, Caspase-3/7 activity was significantly decreased in cells transfected with DUX4 and U6.miDUX4.405, H1.MIR675 and CMV.H19 (49 ± 1%, 34 ± 2% and 24 ± 2%, respectively; P < 0.0001). Two-way ANOVA followed by Dunnett’s multiple comparison tests were performed for statistical analyses. Results reported as mean relative luminescence units (RLU) ± SEM ( N = 3 independent experiment). Source data are provided as a Source data file. Full size image Prior studies showed that DUX4 activates apoptosis in HEK293 cells, which can be measured by activation of Caspase-3/7 [9] , [13] . Thus, to confirm the cell viability assay, we performed a second co-transfection experiment using Caspase-3/7 assay as an outcome measure for apoptosis. Cells co-transfected with DUX4 and U6.milacZ showed a 2.2 ± 0.1-fold increase ( P < 0.0001, ANOVA, N = 3) in Caspase 3/7 activity compared to the Caspase-3/7 activity of mock-transfected (No DUX4 ) cells, indicating an increase in apoptosis. However, U6.miDUX4.405, H1.MIR675 and CMV.H19 reduced Caspase 3/7 activity in cells co-transfected with CMV.DUX4 by 49 ± 1%, 34 ± 2%, and 24 ± 2% respectively ( P < 0.0001, ANOVA, N = 3 for all three conditions) (Fig. 4b ). In addition to Caspase activation, DNA damage is another feature of apoptosis. Indeed, DUX4 causes DNA damage that can be visualized and quantified using an alkaline comet assay (single cell electrophoresis) [36] , [37] . To corroborate the findings from the Caspase-3/7 assay, we performed comet assays to assess DUX4-mediated DNA damage in the presence and absence of miR-675 . To do this, we co-transfected HEK293 cells with plasmids expressing DUX4 and a negative control U6.milacZ; DUX4 and H1.MIR675 ; or DUX4 and U6.miDUX4.405 positive control (Fig. 5a ). Additional controls included mock-transfected cells or cells transfected with a plasmid expressing our previously described, non-toxic DUX4.HOX1 construct that contains mutations in the first DNA binding domain [13] . In cells co-expressing DUX4 and miLacZ, DNA damage was evident by abundant DNA comet tails representing DNA fragments migrating away from cell nuclei (Fig. 5a ). In these cells, the tail moment reached an average of 30 ± 9 µm. In contrast, cells lacking DUX4 or expressing the non-toxic DUX4.HOX1 mutant showed no DNA fragmentation with an average tail moment of 0.67 ± 0.15 µm and 0.28 ± 0.10 µm, respectively. Importantly, co-expression of DUX4 with either miDUX4.405 positive control or H1.MIR675 prevented DUX4-associated DNA fragmentation as the average tail moment reached 5 ± 4 µm for both constructs (~77% reduction when compared to DUX4 + milacZ transfected cells). These results confirmed that DUX4 inhibition by the miDUX4.405 positive control and miR-675 protected cells from apoptosis. Fig. 5: miR-675 protects cells from DUX4-induced DNA damage and transactivation. a Alkaline comet assay using HEK293 cells co-transfected with DUX4 and U6.milacZ, H1.MIR675, U6.miDUX4.405, or negative controls, including the non-toxic DUX4.HOX1 mutant. Comet-like tails in electrophoresed cells indicate DNA damage. To quantify DNA damage, cells were stained with SYBR green fluorescent dye to detect DNA fragments and Tritek CometScore software was used to analyze 10 images of randomly selected non-overlapping cells from two independent replicates. In each image, the average tail moment was calculated (tail length × percent tail DNA) from 30 to 60 nuclei. Mean tail moment was 30 ± 9 µm in DUX4 -expressing cells treated with the miLacZ negative control, while negative controls showed no DNA damage (0.67 ± 0.15 µm and 0.28 ± 0.10 µm, for No DUX4 or DUX4.HOX1, respectively). In contrast, U6.miDUX4.405 and H1.MIR675 protected cells from DUX4-induced DNA damage (mean tail moment of 4.75 ± 4.25 µm and 5.11 ± 4.38 µm, respectively). Data in graph represent the mean tail moment (µm) ± SEM of two independent transfection replicates, repeated with similar results. b MiR-675 reduced DUX4 transactivation function in a DUX4-activated GFP reporter assay. HEK293 cells were co-transfected with DUX4 and either U6.milacZ, CMV.H19 or H1.MIR675, as well as a DUX4-activated GFP reporter (DUX4 Rep), which contains five DUX4-specific binding sites [38] . Mean fluorescence intensity (MFI) was measured using flow cytometry. Cells co-transfected with DUX4 , U6.milacZ and the DUX4-activated GFP reporter showed a MFI of 62744 ± 2040, while CMV.H19 or H1.MIR675 reduced GFP expression by 49 ± 2% (32148 ± 865 MFI; P < 0.0001) and 57 ± 2% (26667 ± 930 MFI; P < 0.0001), respectively. One-way ANOVA followed by Dunnett’s multiple comparison tests were performed for statistical analyses. Values are given as mean MFI ± SEM ( N = 3 independent experiment). Source data are provided as a Source data file. Full size image miR-675 inhibits transactivation of a DUX4-responsive reporter DUX4 binds DNA and transactivates numerous target genes involved in pathways including oxidative stress and cell death, among others. To investigate more directly the ability of miR-675 and its precursor H19 to inhibit DUX4 transactivation activity, we utilized a previously described reporter construct containing five DUX4-specific binding sites upstream of GFP [38] . We co-transfected HEK293s with the DUX4-responsive GFP reporter and plasmids expressing DUX4- and either milacZ , H19 , or miR-675 , then measured mean GFP fluorescence intensity (MFI) using flow cytometry (Fig. 5b ). GFP MFI was reduced 49 ± 2% and 57 ± 2% in cells expressing H19 or miR-675 , compared to cells treated with the U6.miLacZ negative control (Fig. 5b ). Endogenous miR-675 targets DUX4 sequences in human FSHD myotubes To this point in our study, we used transfected HEK293 cells to test the hypothesis that miR-675 inhibits DUX4 expression. Although HEK293s hold several advantages for this type of work, they do not normally express polyadenylated DUX4 or miR-675 and are not muscle cells. As a next step, we sought to determine if miR-675 could regulate DUX4 expression in human muscle cells that naturally expressed DUX4 and/or miR-675 . Accomplishing this required two new sets of reagents: (i) antagomirs, which are small oligonucleotides used to silence endogenous miRNAs; and (ii) three human myoblast cell lines, including two from FSHD-affected patients (15A and 17A) that express sporadic and low levels of endogenous DUX4 ; and an unaffected, DUX4 -negative control myoblast line (15V) [39] , [40] . Prior to using these reagents experimentally, we opted to first validate their functionality by confirming miR-675 and DUX4 gene expression in 15A, 17A, and 15V cells (Supplementary Note 5 , Supplementary Fig. 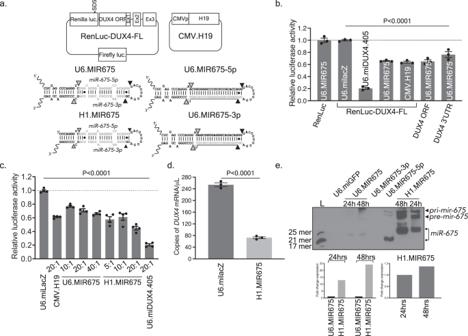Fig. 1:miR-675targets theDUX4 ORFand3′UTR. aRenLuc-DUX4-FL dual-luciferase reporter and CMV.H19 constructs, and U6.MIR675, H1.MIR675, U6.MIR675-3p, and U6.MIR675-5p miRNAs. RenLuc-DUX4-FL containsDUX4 ORFand3′UTRsequences fused toRenillaluciferase after the stop codon. Exons 1–3 are indicated (Ex1,2,3). *SD5 indicates silent mutation of a cryptic splice donor inRenillaluciferase. Firefly luciferase is used as transfection control.bU6.MIR675 reduced relativeRenillaluciferase activity in constructs containing full-lengthDUX4,DUX4ORF only, orDUX43’ UTR only (35 ± 3%, 34 ± 2%, and 24 ± 5%, respectively;P< 0.0001).H19reduced relativeRenillaluciferase activity from the RenLuc-DUX4-FL by 36 ± 2% (P< 0.0001). All readings were normalized to Firefly luciferase and then to the milacZ negative control. U6.MIR675 did not reduce relativeRenillaluciferase activity from the non-targeting RenLuc control plasmid (RenLuc). The U6.miDUX4.405 positive control is a published artificial microRNA with robustDUX4silencing activity. Data indicate mean luciferase activity ± SEM (N= 3 independent experiments).cRelativeRenillaluciferase activity was reduced in a dose-dependent manner by twomiR-675constructs: U6.MIR675 and H1.MIR675. Molar ratios of miRNA to reporter plasmid are indicated and data normalized to the miLacZ negative control. U6.MIR675 significantly reduced relativeRenillaluciferase activity by 23 ± 3% (10:1 ratio), 29 ± 3% (20:1), and 34 ± 3% (40:1). H1.MIR675 performed better at lower doses, reducing relativeRenillaluciferase activity by 42 ± 4%, 39 ± 5%, and 55 ± 3%. All samples were significantly different from the miLacZ control (P< 0.0001). Data represent mean normalizedRenillaluciferase activity ± SEM (N= 4 independent experiments).dDroplet digital PCR (ddPCR). H1.MIR675 significantly reducedDUX4mRNA levels by 71 ± 2% (P< 0.0001, ANOVA,N= 3) compared to the miLacZ negative control, 48 h following transfection of HEK293 cells with a 1:3 ratio of CMV.DUX4-FL/CMV.eGFP and H1.MIR675. Results represent the average absoluteDUX4mRNA concentration (copies/µL) ± 95% poisson confidence interval. Data represent mean relative concentration (copies/μL) ± SEM (N= 3 independent experiments). Forb–d, One-way ANOVA followed by Dunnett’s multiple comparison tests were performed for statistical analyses.eNorthern blot using RNA extracted from HEK293 cells transfected with the indicated expression plasmids. U6.miGFP is a negative control. Source data are provided as a Source data file. 10 and Supplementary Table 1 ). We also empirically tested the impact of inhibiting miR-675 with an antagomir on Renilla luciferase activity encompassing in its 3′UTR a perfect miR-675-5p target site (RenLuc-miR-675R), and on CDC6 , a known miR-675 target gene (Supplementary Note 5 , Supplementary Figs. 11 and 12 ). We next examined the ability of miR-675 inhibition to de-repress wild-type and mutant DUX4 sequences. We again employed the dual luciferase reporters, where one plasmid contained full-length wild-type DUX4 sequences (DUX4-FL) and a second contained miR-675 -resistant mutations (DUX4ORF-mir675Res). These plasmids were co-transfected into 15V unaffected and 15A FSHD myoblasts along with miR-675 or negative control antagomirs (anti-miR-675 or anti-miR-ctrl). The presence of anti-miR-675 significantly increased the relative Renilla luciferase activity from RenLuc-DUX4-FL in 15V cell lines by 1.5 ± 0.1-fold ( P < 0.0001, ANOVA, N = 3) and in 15A cell lines by 2.1 ± 0.1-fold ( P < 0.0001, ANOVA, N = 3), while the negative control antagomir had no impact (Fig. 6a ). These results suggested that miR-675 was able to silence DUX4 sequences via RNAi. To confirm these results, we performed the same experiment using Renilla luciferase tagged with miR-675 -resistant DUX4 sequences. In all cases, cells expressing the miR-675 -resistant plasmid produced more luciferase activity, compared to their counterparts expressing Renilla luciferase fused to the wild-type DUX4 sequence (Fig. 6a ). Nevertheless, we still saw de-repression when anti-miR-675 was transfected along with the miR-675 resistant luciferase plasmid (1.8- to 1.3-fold increase in luciferase activity, P < 0.0001 and P = 0.0078, respectively in 15V and 15A cells compared to cells that received the anti-miR-ctrl). These results suggested that miR-675 was still capable of mediating some inhibition, albeit weaker, on the resistant Renilla luciferase- DUX4 fusion sequence by binding to the remaining, non-mutated, lower affinity target sites on the DUX4 sequence. Fig. 6: Endogenous miR-675 targets DUX4 and prevents expression of DUX4-responsive biomarkers in 15A FSHD-affected human myotubes. a Dual-luciferase assay in 15V Ctrl and 15A FSHD myoblasts. DUX4 -tagged Renilla luciferase (RenLuc-DUX4-FL) or miR-675 -resistant Renilla luciferase (RenLuc-DUX4 ORF-miR-675Res) plasmids were co-transfected with 300 nM anti-miR- ctrl or anti-miR-675 into 15V and 15A cells. Relative Renilla luciferase activity was measured at 48 h. Addition of DUX4 sequences to the end of Renilla luciferase caused a significant decrease in relative luciferase activity in both cell lines (compare RenLuc-DUX4-FL to RenLuc only; mean 41 and 65% reduction in luciferase activity in 15V and 15A cells respectively; ( P < 0.0001). Transfection of the anti-miR-675 caused a 1.5–2.0-fold increase of luciferase activity in the DUX4-FL-tagged Renilla luciferase construct, compared to cells that received the anti-miR-ctrl ( P < 0.0001). All data represent mean normalized Renilla luciferase activity ± SEM ( N = 3 independent experiments). Two-way ANOVA followed by Tukey’s multiple comparison tests were performed for statistical analyses. b Gene expression results in 4-day differentiated 15A FSHD cells transfected with 300 nM anti-miR-675 or an anti-miR -ctrl. Left panels, QPCR. Treatment with anti-miR-675 decreased mean miR-675-5p levels 23 ± 2-fold ( P < 0.0001) and caused a 3-fold increase of DUX4 -responsive biomarkers TRIM43 and KHDC1L 3 ( P < 0.0001). Results were reported as gene expression (∆∆Cq) ± SEM ( N = 3 independent experiments), normalized to 15A FSHD cells transfected with anti-mir-ctrl . Right panels, ddPCR results for endogenous DUX4 , miR-675 , and TRIM43 using RNA acquired from a similar set of anti-mir transfection experiments. Treatment with anti-miR-675 decreased mean miR-675-5p levels 12 ± 1-fold ( P = 0.0118), while DUX4 and TRIM43 expression increased 3.4 ± 0.6-fold ( P < 0.0001) and 1.9 ± 0.3-fold ( P = 0.0074), respectively. Results were reported as the mean absolute DUX4 , miR-675-5p , or TRIM43 concentration (copies/µL) ± 95% poisson confidence interval normalized to human RPL13A . Data represent mean relative concentration (copies/µL) ± SEM ( N = 3 independent experiments) normalized to cells transfected with anti-mir-ctrl . For QPCR and ddPCR, two-way ANOVA followed by Sidak’s multiple comparison tests were performed for statistical analyses. Source data are provided as a Source data file. Full size image Using QPCR, we found that the anti-miR-675 antagomir significantly reduced miR-675-5p by an average of 23 ± 2-fold ( P < 0.0001, ANOVA, N = 3 independent experiments) (Fig. 6b ). In addition, 15A FSHD cells transfected with anti-miR-675, and subsequently differentiated for 4 days, had levels of the DUX4-responsive biomarkers TRIM43 and KHDC1L increase by 3-fold when compared to cells that received the anti-mir control ( P < 0.0001, ANOVA, N = 3 independent experiments). In a second anti-miR study in differentiated 15 A cells, we measured DUX4 , miR-675-5p , and TRIM43 expression using ddPCR. MiR-675-5p expression significantly decreased (12 ± 1-fold; P = 0.0118, ANOVA, N = 3 independent experiments), while endogenous DUX4 and the DUX4-responsive biomarker TRIM43 significantly increased by 3.4 ± 0.6-fold ( P < 0.0001, ANOVA, N = 3 independent experiments) and 1.9 ± 0.3-fold ( P = 0.0074, ANOVA, N = 3 independent experiments), respectively (Fig. 6b ). These data are consistent with expected results arising from inhibiting a DUX4 inhibitor (anti-miR-675 =↓ miR-675 =↑ DUX4 = ↑ DUX4 -responsive biomarkers) (Fig. 6 ). Importantly, using the most comprehensive atlas of miRNA-target interactions (miRwalk2.0), miR-675 was not predicted to target TRIM43 nor KHDC1L , suggesting that their expression changes indirectly resulted from miR-675 knockdown of DUX4 [41] (Supplementary Data 2 , 3 , and 4 ). Endogenous miR-675 regulates DUX4 protein expression in myotubes To evaluate the effect of endogenous miR-675 on the levels of transfected DUX4 , we performed western blot on proteins extracted from 15 A FSHD cells transfected with V5-tagged DUX4-FL or miR-675 -resistant DUX4 (DUX4-miR-675Res) expression plasmids with and without anti-miR-675. After four days of differentiation, we detected minimal amounts of DUX4.V5 protein in one of the three replicates transfected with DUX4 alone (Fig. 7a and Supplementary Fig. 13 ). No DUX4 signal was found in the other two replicates. We found increased DUX4 signal upon adding anti-miR-675 (Fig. 7a and Supplementary Fig. 13 ). DUX4 signal was notably higher in cells transfected with the miR-675 -resistant DUX4 construct, and some additional de-repression was evident in cells treated with anti-miR-675, suggesting that miR-675 could still repress DUX4 , perhaps utilizing the minor binding sites we did not mutate in the resistant constructs. The difference in DUX4 protein levels in cells transfected with the wild-type and miR-675 -resistant construct was surprisingly large. We engineered the miR-675 -resistant DUX4 construct to contain silent mutations in the TS780 miR-675 binding site and to not contain its 3’UTR sequence and, therefore, expresses wild-type DUX4 protein. To rule out the possibility that unexpected differential toxicity could contribute to the differences in DUX4 protein levels arising from the two constructs, we used Caspase-3/7 assay to confirm that both sequences were capable of producing cell death (Supplementary Note 6 and Fig. 7a ). As a result, DUX4 levels in the western blots correlated with Caspase-3/7 activation, as cells with the highest amounts of DUX4 had increased levels of cell death. In this Caspase-3/7 assay, we also showed that the inhibition of miR-675 with anti-miR-675 increased cell death in 15A FSHD myotubes. Fig. 7: Endogenous miR-675 targets DUX4 and prevents DUX4-induced toxicity in 15A FSHD-affected human myotubes. a Western blots. V5-epitope tagged wild-type or miR-675-resistant DUX4 plasmids were transfected into 15A FSHD myotubes co-treated with anti-miR-675 or anti-miR-ctrl. DUX4 expression plasmids also contained a separate CMV.eGFP reporter that was used as a transfection control and western blot normalizer. Proteins were harvested 4 days after differentiation, followed by western blot using antibodies to detect V5, eGFP, and β-actin. DUX4-V5 signal was absent in mock-transfected cells and below the level of detection in cells transfected with wild-type DUX4 and the anti-miR-ctrl. However, DUX4.V5 signal was detected in cells co-transfected with wild-type DUX4 and anti-miR-675. Increased DUX4 protein was evident in cells transfected with miR-675 -resistant DUX4, using both anti-miR-675 and anti-miR-ctrl. Two additional western blot replicates were performed (Supplementary Fig. 13 ). In Caspase-3/7 assay, anti-miR-675 transfection increased Caspase-3/7 activity in 15A cells by 3.2 ± 0.3-fold compared to those treated with anti-miR-ctrl ( P < 0.0001), while with DUX4 full-length or miR-675-resistant DUX4 expression plasmids increased Caspase-3/7 activity by 5.6 ± 0.4-fold and 10.6 ± 0.8-fold, respectively ( P < 0.0001). Results were reported as the mean Caspase 3/7 activity (RLU) ± SEM ( N = 3 independent experiments). One-way ANOVA followed by Tukey’s multiple comparison tests were performed for statistical analyses. b Immunofluorescence (IF) to detect endogenous DUX4 protein in 4-days differentiated 15A FSHD myotubes transfected with 150 nM of anti-mir-ctrl or anti-miR-675. Cells were stained with a 1:100 dilution of DUX4 antibody (mouse mAB 9A12) followed by fluorescence-labeled secondary antibodies. Myotubes treated with anti-mir- ctrl and anti-miR-675 had an average of 0.11 ± 0.02, and 0.77 ± 0.21 DUX4 + per 10,000 nuclei, respectively. Myotubes treated with anti-miR-675 had their number of DUX4+  nuclei increase by 7 ± 2-fold ( P = 0.0369). The graph shows quantification of number of DUX4 + per 10,000 nuclei. Results were reported as DUX4 + nuclei per 10,000 nuclei ± SEM ( N = 3 independent experiments, repeated with similar results with two technical replicates per experiment). Unpaired two-tailed t test was performed for statistical analyses. Source data are provided as a Source data file. Full size image Next, to evaluate the effect of endogenous miR-675 on endogenous DUX4, we transfected 15A FSHD myoblasts with anti-miR-675 or anti-miR -ctrl, differentiated cells for 4 days, and then used immunofluorescence to detect DUX4 protein. Anti-miR-675-treated myotubes showed a 7 ± 2-fold increase in DUX4 + nuclei compared with myotubes treated with anti-miR-ctrl ( P = 0.0369, unpaired two-tailed t -test, N = 3 independent experiments) (Fig. 7b ). Taken together, these results suggested that the endogenous miR-675 targeted the transfected or endogenous DUX4 sequence and reduced DUX4 protein levels, while DUX4 expression and DUX4-induced toxicity were increased upon miR-675 inhibition with the anti-miR-675 antagomir. AAV-based miR-675 gene therapy reduces DUX4 expression and counteracts DUX4-induced toxicity in a DUX4 mouse model Our results to this point suggested that miR-675 upregulation might be useful as an FSHD therapy. To test this idea, we used two strategies: (i) AAV.MIR675-based gene therapy in a DUX4 -expressing mouse model; and (ii) drug-based therapy aimed to increase miR-675 expression in FSHD patient cells. For gene therapy, we packaged miR-675 expression cassettes into serotype 6 self-complementary adeno-associated viral vectors (scAAV6), which are myotropic. Unfortunately, the original H1.MIR675 sequence we used for in vitro studies caused histopathology when delivered to wild-type C57BL/6 mouse muscle in vivo with AAV (Supplementary Fig. 14 ). The inability to safely translate a microRNA expression cassette from an in vitro to in vivo system was not unprecedented [29] , and could result from misfolding of 5′ and 3′ sequences flanking the pre-miRNA, leading to suboptimal processing in vivo. We, therefore, optimized these sequences to improve folding, while maintaining the natural pre-mir-675 sequences, and identified a construct capable of producing mature miR-675 without causing in vivo toxicity in mouse muscle ( optimization manuscript in preparation ). We next tested the ability of this new vector (scAAV6.MIR675) to protect mouse muscles from DUX4-induced damage in vivo using an AAV-based DUX4 model similar to one we previously described, but containing the DUX4 3′UTR sequences in addition to a V5 epitope-tagged DUX4 open reading frame (ORF) [13] , [42] . We used this construct because miR-675 possesses target sites within the DUX4 ORF and 3′UTR (Fig. 2 ). We co-injected 5 × 10 10 scAAV6.MIR675 particles, or 5 × 10 10 particles of the non-targeting AAV.miLacZ control, with a 3 × 10 9 AAV6.CMV.DUX4-FL, into C57BL/6 mouse TA muscles (Fig. 8 and Supplementary Fig. 15 ). We then assessed DUX4-induced muscle histopathology, and measured the expression of DUX4 and DUX4-responsive mouse biomarkers. Fig. 8: miR-675 protects mouse skeletal muscles from DUX4-induced muscle damage. a H&E staining, central nuclei counts, and gene expression analysis of AAV-injected adult mouse (C57BL/6) tibialis anterior (TA) muscles 2 weeks after IM delivery of indicated vectors. Images show 10 µm H&E-stained cryosections at high (×20) and low power (×4). To visualize the breadth of lesions on low-power images, fibers with central nuclei (CN), degeneration or inflammation were intentionally shaded with a purple digital overlay. Control-treated, DUX4-expressing muscles show histopathological evidence of degeneration, including myofibers with inflammatory infiltrates, central nuclei, and variable fiber size (top left). In contrast, the AAV6.MIR675 vector protected muscles from DUX4-induced damage at the same time point. High-power photos show representative images at indicated vector dosages. Images are representative of the following N’s: AAV6.DUX4-FL + AAV6.MIR675, N = 8 TA muscles; AAV6.DUX4-FL + negative control (AAV6.miLacZ or AAV6.eGFP), N = 5 TA muscles; No DUX4 , i.e., AAV6.miLacZ + AAV6.MIR675, N = 3 TA muscles. CN counts from 20x H&E-stained TA muscle serial sections. (Left) AAV6.MIR675-treated muscles showed 81 ± 6% fewer myofibers with central nuclei compared to the negative control-treated muscles (**** P = 0.0004, two-tailed unpaired t -test). Droplet digital PCR (ddPCR) showed significant 56 ± 12% reduction in DUX4 mRNA in AAV6.MIR675-treated versus negative control-treated TA muscles ( N = 8 miR-675 -treated and N = 5 negative control-treated mice; unpaired two-tailed t test, * P = 0.01). (Middle) ddPCR of miR-675 and DUX4 -responsive mouse biomarkers in AAV6.MIR675 treated and un-treated TA muscles. Trim36 and Wfdc3 expression was reduced by 88 ± 4% (*** P = 0.0004) and 57 ± 13% (* P = 0.011), respectively. Results reported as average absolute DUX4, hsa-miR-675-5p, Trim36 or Wfdc3 copies/µL ± 95% poisson confidence interval ± SEM, normalized to mmu-Rpl13A . For miR-675-5p , Wfdc3 , and Trim36 , one-way ANOVA followed by Tukey’s multiple comparison tests were performed for statistical analyses. (Right) Western blots using proteins from injected TA muscles (uncropped western blots in Supplementary Fig. 16 ). Anti-V5 epitope antibodies were used to detect V5-tagged DUX4, with α-tubulin used as a loading control. b High-power photos show representative images at indicated vector dosages of N = 8 TA co-injected with AAV6.MIR675 or negative control vector with AAV6.DUX4-FL. H&E or immunofluorescence staining of 10 µm cryosections, using antibodies to detect DUX4 (V5, red) or DAPI (nuclei, blue). White arrows indicate myonuclei showing DUX4-V5 signal (red). Green arrows indicate degenerating myofibers containing some red signal in the cytoplasm, potentially indicating nuclear breakdown and DUX4 leaking into the cytoplasm [21] . All Ns were repeated with similar results. Full size image Muscles co-injected with AAV.milacZ and AAV.CMV.DUX4-FL showed obvious and widespread histopathology, with mononuclear cell infiltration, and an abundance of centrally nucleated myofibers (mean 24 ± 5%), a feature which indicates muscle damage and repair. In contrast, muscles co-injected with scAAV6.MIR675 with and without AAV.CMV.DUX4-FL were histologically normal (mean 5 ± 1% centrally nucleated myofibers), demonstrating that scAAV6.MIR675 is not toxic to normal mouse muscle and, importantly, can counteract DUX4-induced muscle damage in vivo (Fig. 8 and Supplementary Fig. 15 ). Consistent with the histopathological protection, compared to controls, scAAV6.MIR675-injected muscles also showed significantly reduced expression of DUX4 (56 ± 12%, P = 0.01) and the DUX4 -responsive biomarkers Trim36 and Wfdc3 , (88 ± 4%, P = 0.0004; and 57 ± 13%, P = 0.011, respectively), as determined by ddPCR (Fig. 8a ). We also measured V5-tagged DUX4 protein levels using western blot, and found less DUX4 protein in AAV.DUX4-injected TA muscles co-injected with scAAV6.MIR675 compared to AAV.miLacZ controls (Fig. 8a and Supplementary Fig. 16 ). Finally, we stained TA muscle sections from co-injected animals with a red fluorophore-tagged anti-V5 antibody to detect V5-tagged DUX4 protein, and found reduced or absent DUX4 protein expression in TA muscle sections treated with AAV.CMV.DUX4-FL and scAAV6.MIR675, compared to those that received identical amounts of AAV.CMV.DUX4-FL and non-targeting miLacZ control vectors (Fig. 8b and Supplementary Fig. 17 ). As previously reported using the AAV.DUX4 model, some damaged muscle fibers showed cytoplasmic staining of DUX4 protein. We speculate this is due to nuclear membrane leakage in dying myofibers (Fig. 8b ). Small molecule upregulation of miR-675 reduces DUX4 and TRIM43 expression in FSHD patient myotubes Gene therapy has the potential to provide stable and long-lasting expression of a therapeutic microRNA product, such as miR-675 . However, there are also potential risks; if a vector-delivered microRNA causes unforeseen off-target effects, it is currently not possible to turn it off or tune down expression. We therefore also pursued an alternative strategy that, to our knowledge, has never been previously attempted. Specifically, we sought to increase endogenous miR-675 expression in FSHD affected muscle cell lines using a drug-based therapy, which would be tunable and potentially stopped if untoward events arose. Having identified miR-675 as a strong endogenous regulator of DUX4 , we decided to search within previously published gene expression data for small molecules that increase miR-675 expression or its H19 precursor. We identified three candidates (β-estradiol, combination of β-estradiol + medroxyprogesterone acetate (MPA), and melatonin) that were shown to increase miR-675 expression in various models but had not been tested in the cell models we used here, HEK293s and human myotubes [43] , [44] , [45] . We first confirmed the system in transfected HEK293s (Supplementary Note 7 , Supplementary Data 5 , and Supplementary Fig. 18 ). We then tested the effect of the three molecules on the expression of endogenous miR-675-5p , DUX4 and DUX4-responsive biomarker, TRIM43 in 15A, 18A, and 17A FSHD differentiated muscle cell lines (myotubes), which express different levels of DUX4 (15A < 18A < 17A) (Fig. 9 ) [39] . All three molecules were added to myotubes on the 4th day of differentiation and cells were harvested 24 h later. 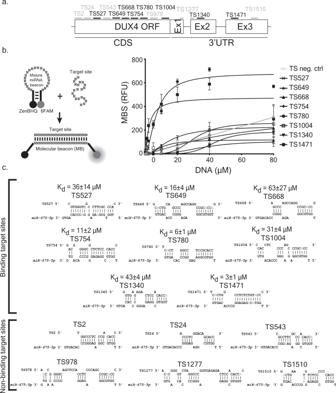Fig. 2:miR-675-5ptargets multiple binding sites in theDUX4 ORFand3′UTR. aSchematic ofDUX4sequence showing predicted target site (TS) positions formiR-675-5p.b(Left) Molecular beacon binding assay used to determinemiR-675-5pbinding toDUX4. Unbound, the molecular beacon folds into a stem loop structure that brings the ZenBHQ quencher in close proximity to a the 6FAM fluorophore, thereby preventing 6FAM fluorescence. We incorporated the mature sequence ofmiR-675-5pin the MB loop sequence. Hybridization of the MB to a complementary DUX4 target sequence separates the fluorophore and quencher, allowing fluorescence emission, which is quantified as a measure of binding. (Right) The graph shows binding of the maturemiR-675-5pmolecular beacon to target sites shown in (a).miR-675-5pbound 8DUX4target sites (6 in the ORF and 2 in the 3′UTR). Six predicted TS did not bind tomiR-675-5p(Supplementary Fig.3band Supplementary Data1for TS position and sequence). The TS neg. ctrl is a random sequence. Curves are fit into one site-specific binding with Hill slope equation. Each data point represents mean ± SD (N= 3 independent experiments).cBase-pairing ofmiR-675-5pand predictedDUX4target sites used in the molecular beacon assay. The binding affinity (Kd) ofmiR-675-5pmolecular beacon to each target site was determined by subtracting background fluorescent signal from the molecular beacon signal (MBS), expressed in relative fluorescent units (RFU). TheKdcorresponds to the TS concentration (μM) required to reach half of maximum fluorescence. We generated RNA “mimic” bases in themiR-675-5p:TS pair and replaced “G” nucleotides with “A” nucleotides (in gray) whenever the “G” is facing a “T”29. Source data are provided as a Source data file. In 15A myotubes, all three molecules triggered an increase in miR-675 expression (Supplementary Table 2 and Fig. 9a ). DUX4 and TRIM43 mRNA expression significantly decreased in 15A myotubes treated with β-estradiol+MPA or melatonin. However, the treatment with β-estradiol alone did not trigger a significant decrease in TRIM43 expression (Supplementary Table 2 and Fig. 9a ). In 17A and 18A myotubes, β-estradiol, β-estradiol+MPA, or melatonin triggered a significant increase in miR-675 expression that was associated with significant decreases in DUX4 and TRIM43 mRNA expression (Supplementary Table 2 and Fig. 9a ). Importantly, control experiments suggested that these drugs did not directly reduce TRIM43 or significantly impact myoblast differentiation, thereby supporting our hypothesis that RNAi mediated by small molecule upregulation of miR-675 could reduce DUX4 and indirectly decrease a DUX4-responsive biomarker in FSHD muscle cells (Supplementary Note 8 and 9 and Supplementary Fig. 19 ). Fig. 9: β-estradiol, medroxyprogesterone acetate (MPA), and melatonin increased miR-675 expression and reduced the expression of DUX4 and DUX4-responsive biomarker TRIM43 in 3 FSHD affected myotube lines. a Droplet digital PCR (ddPCR) to measure miR-675-5p , DUX4 , and TRIM43 levels in 15A, 17A, and 18A FSHD affected myotubes, 5 days after differentiation. We added two drugs individually (i.e., β-estradiol and melatonin) or as a combination (β-estradiol + MPA) on the 4th day of differentiation. All treatments were compared to ethanol (vehicle) treated control cells. N = 6 independent experiments for 15A and N = 3 for 17A and 18A. * P = 0.05. ** P = 0.01. *** P = 0.001. Results were reported as the average absolute DUX4, miR-675-5p, or TRIM43 concentration (copies/µL) ± 95% poisson confidence interval normalized to hsa-RPL13A . Data represent mean relative concentration (copies/µL) ± SEM ( N = 3–6 independent experiments). b Immunofluorescence on 18 A FSHD affected myotubes following 5 days of differentiation, and 24 h post-treatment with 20 µM of β-estradiol, β-estradiol, and MPA or Melatonin. DUX4 protein was detected with 1:100 of DUX4 antibody (mouse mAb 9A12). Myotubes mock-treated with 100% ethanol had an average of 12.8 ± 0.8 DUX4 + per 10,000 nuclei. Treatment with β-estradiol, β-estradiol and MPA or Melatonin reduced DUX4 + nuclei per 10,000 in myotubes (8.3 ± 0.4, 6.7 ± 0.5 and 6.0 ± 0.4 DUX4+ nuclei per 10,000, respectively; *** P = 0.0010; *** P = 0.0001; **** P < 0.0001). Results represent mean DUX4 + nuclei per 10,000 nuclei ± SEM ( N = 3 independent experiments, repeated with similar results with two technical replicates per experiment). For a , b one-way ANOVA followed by Dunnett’s multiple comparison tests were performed for statistical analyses. Full size image Finally, to assess the effect of the three molecules on DUX4 protein levels, we performed an immunofluorescence assay in 18A FSHD affected myotubes differentiated for 4 days [39] . Myotubes were treated with β-estradiol, β-estradiol, and MPA, melatonin, or vehicle, and then stained for DUX4 protein 24 h later using a DUX4-targeting antibody (mouse mAb 9A12, 1:100 dilution). Similar to previous reports, DUX4 protein was rare, as mock-treated myotubes had an average of 12.8 ± 0.8 DUX4 + per 10,000 nuclei [39] . However, DUX4+ nuclei decreased in myotubes treated with β-estradiol, β-estradiol and MPA or melatonin by 35 ± 5%, 48 ± 5%, and 54 ± 4%, respectively (8.3 ± 0.4, 6.7 ± 0.5, and 6.0 ± 0.4 DUX4 + nuclei per 10,000) (Fig. 9b ). The discovery of RNAi and mammalian microRNAs over 20 years ago added to the diversity of functions that RNA molecules play in gene expression, and importantly, provided new tools to develop powerful gene silencing therapies. Most RNAi therapy strategies use artificial RNAi triggers, like siRNAs, shRNAs, or microRNA shuttles, which are engineered to contain ~22 nucleotide (nt) of perfect sequence complementarity with a target gene [46] . Indeed, to date the only three FDA-approved RNAi drugs, Alnylam’s Patisiran, Oxlumo and Givlaari, utilize an engineered siRNA approach to inhibit disease genes. Similarly, our published DUX4 -targeting gene therapy strategy utilizes an engineered microRNA shuttle system in which the mature sequences have perfect 22 nt base-pairing with the DUX4 transcript. The main advantage of this approach is potency; in general, greater complementarity between a target transcript and a mature microRNA yields greater gene silencing, often >90%. In contrast, most natural microRNAs have several mismatches with their gene targets, leading to relatively weak or modest silencing. Despite the advantages of using an engineered system, some studies have described using natural microRNA sequences as potential treatments for disease, such as mir-26a gene replacement in a mouse model of mir-26a -deficient hepatocellular carcinoma [47] . In all cases described to date, these natural microRNA sequences were exogenously delivered as oligonucleotides or using gene therapy vectors. Here, we also pursued a strategy to use a natural microRNA— miR-675 —for therapeutic purposes. In addition to using a traditional gene therapy approach to deliver miR-675 (Fig. 8 ), we also developed a small molecule-based strategy that, to our knowledge, had never been described before for any disease (Fig. 9 ). Specifically, we pursued a simple therapeutic model based on two main ideas: (i) endogenous microRNA gene expression can change in response to small molecule treatments; (ii) if natural DUX4 -targeting microRNAs exist, their upregulation should serve to decrease DUX4 expression via the RNAi pathway. By combining these two ideas, we reasoned that an FSHD therapy could be developed by using small molecules to increase expression of natural microRNAs that target DUX4 for degradation within the cell. Thus, our approach was target-based and relied upon a known mechanism of DUX4 inhibition with RNAi. From the outset, there were two practical problems with this strategy: (i) there were no microRNAs known to regulate DUX4 ; and (ii) even if we could identify a DUX4 -targeting microRNA, we were not certain if the appropriate transcriptomic data existed to support small molecule upregulation of such a candidate microRNA. We thus began by working to determine if any natural microRNAs functioned to inhibit DUX4 . Prior gene expression studies reported microRNAs that were differentially expressed in FSHD cells compared to controls, but the biological significance of any of the putative FSHD-related miRNAs remained unclear and no DUX4 -targeting miRNAs were identified in any of these studies [48] , [49] , [50] , [51] , [52] , [53] . In our study, differential gene expression in FSHD was not part of our screening criteria when identifying miRNA candidates. Indeed, we only considered one question to determine if a specific miRNA was potentially important—does it target DUX4 ? We selected 24 putative DUX4 -targeting miRNAs from two different bioinformatics algorithms for empirical testing. This represented 1.3% of the 1917 known human miRNAs. We then used a battery of empirical tests to confirm—or mostly, refute—the ability of these 24 predicted miRNA candidates to silence DUX4 . MiR-675 was the only one that regulated DUX4 , but did so powerfully and consistently using numerous different assays, and having multiple binding sites in both the ORF and 3′ UTR of the DUX4 mRNA. This single miRNA represents 0.05% of all known human miRNAs, and it is possible that miR-675 is not the only DUX4 -targeting miRNA—just the first identified. Additional work is required to mine the miRNome for additional DUX4 -targeting microRNAs. In addition to the RNAi mechanism we explored here, nonsense mediated decay (NMD) has also been shown to regulate DUX4 mRNA degradation [54] . This mechanism involves a double-negative feedback loop involving NMD and DUX4 . In this model, NMD normally degrades DUX4 mRNA, but rare transcripts can escape NMD and become translated into DUX4 protein, which causes proteolytic degradation of UPF1, a key component of the NMD process. Thus, DUX4 protein inhibits NMD, thereby allowing local amplification of DUX4 gene expression until enough DUX4 protein is produced to presumably kill the cell. Since translation and RNAi both occur in the cytoplasm, it is possible that miR-675 and the miRNA pathway could target and reduce DUX4 transcripts that escape NMD (Supplementary Fig. 20 ). This has implications for emerging gene silencing therapies for FSHD, which could help to avoid “bursts” of DUX4 expression that escape NMD inhibition. Having identified miR-675 as a DUX4 regulator, we then worked to leverage this finding for therapeutic purposes in FSHD. We first took a gene therapy approach to express miR-675 in DUX4 -expressing mouse muscle, using a strategy similar to the one we developed using artificial microRNAs (Fig. 8 ) [21] , [29] , [33] , [55] . Because miR-675 was almost as potent an RNAi trigger as our artificial microRNA miDUX4.405 , we were not surprised to find that over-expression of AAV-delivered miR-675 prevented DUX4-associated toxicity and suppressed DUX4-responsive biomarkers in mouse muscle. Thus, our data support another avenue for RNAi-based gene therapy of FSHD, using a natural microRNA. Having established proof-of-principle for using miR-675 as a potential therapy for FSHD, we next assessed the possibility of using small molecules to upregulate miR-675 as potential DUX4 -targeting therapeutics, which was the main aim of our study. Prior studies showed that miR-675 was induced with treatment of melatonin, and estrogen alone or in combination with progesterone [43] , [44] , [45] . In this work, we tested melatonin, estrogen (β-estradiol), and progesterone (medroxyprogesterone acetate) analogs on HEK293 cells that usually express very minimal levels of miR-675 , and on three FSHD muscle cell lines expressing low (15A), medium (18A) and high (17A) levels of DUX4 . We confirmed that each of the compounds indeed increased miR-675 in our cell culture systems and operated to decrease DUX4 and the DUX4 -responsive biomarker TRIM43 expression in all cell lines tested (Fig. 9a, b ). Importantly, inhibiting miR-675 with the anti-miR-675 antagomir or preventing its binding to a miR-675 -resistant DUX4 construct (CMV.DUX4 miR-675Res) supported that the three molecules exert their DUX4 inhibitory effect through miR-675 action (Supplementary Fig. 18 ). Additional experiments, whether by testing the 3 molecules on FSHD affected myotubes overexpressing miR-675 (Fig. 9c ), on healthy control myotubes (Supplementary Fig. 19a ) or by assessing their effect on differentiation Supplementary Fig. S19b ), consolidated this proposition. Interestingly, recent evidence showed that miR-675 levels decrease in muscle with age and since FSHD is a progressive disease that tends to worsen with age, it is possible that miR-675 reductions could mechanistically contribute to progression by having reduced inhibitory effects on DUX4 [56] , [57] , [1] , [2] , [3] , [4] . Thus, by re-establishing high levels of miR-675 in aging skeletal muscles, these small molecules could reduce DUX4-induced muscle damage. Interestingly, estrogen or its derivative β-estradiol have been previously linked to FSHD pathogenesis, although the role of FSHD in the disease is not definitive. Some previous reports suggested that estrogen might be protective in FSHD disease, as females were reported to be less severely affected than males and may have persistent worsening of symptoms after childbirth and menopause [58] , [59] , [60] . One study suggested that the beneficial effects of estrogen were mediated by the estrogen receptor (ERβ), which, when activated by estrogen, sequesters the DUX4 protein in the cytoplasm of cells and prevents its toxic effects in nuclei [61] . In contrast to these reports suggesting a protective effect of estrogen, a recent study of FLExDUX4 mice reported that females perform worse than males in some outcome measures [62] . However, we note that ERT2 system used to generate these animals utilizes the anti-estrogen drug Tamoxifen to induce high levels of DUX4 expression, thereby complicating interpretation of the impacts of estrogen on phenotypes in these animals. In addition, a recent clinical study of 85 female FSHD patients did not find a significant correlation between differences in estrogen exposure and disease severity [63] . Interestingly their clinical approach consisted of subtracting periods with high progesterone levels from the reproductive life span so a protective effect caused by interplay with other reproductive hormones, including progesterone, could not be ruled out. Here, our data suggest a mechanism by which estrogen, and/or estrogen and progesterone, could at least partially protect cells from FSHD disease by counteracting DUX4 expression via miR-675 upregulation. Melatonin has been previously identified as a promising drug therapy for neuromuscular diseases due to its anti-inflammatory and antioxidant properties. For this purpose, it was tested in the mdx5Cv Duchenne muscular dystrophy (DMD) mouse model, where it improved muscle function and enhanced the redox status of the muscle [64] . In another study, melatonin prevented the premature senescence of cardiac progenitor cells that occurs in heart diseases. The study revealed that melatonin exerts its effect via the H19 / miR-675 /USP10 pathway in which miR-675 targets the USP10 peptidase, leading to a downregulation of p53 and p21 proteins [43] . Some previous studies suggested a role of p53 in DUX4 toxicity, although this finding has not been universally supported in all systems [5] , [13] , [19] , [65] , [66] , [67] , [68] . Nevertheless, it is possible that in addition to targeting DUX4 , miR-675 could also target the ubiquitous USP10 protein in FSHD skeletal muscles, leading to a better outcome. Finally, miR-675 has been shown to possess the property of enhancing skeletal muscle regeneration and differentiation by targeting and down-regulating the anti-differentiation SMAD transcription factors (SMAD1 and SMAD5) critical for the bone morphogenetic protein (BMP) pathway and the DNA replication initiation factor CDC6 (ref. [27] and Supplementary Fig. 2 , 11b and 12 ). Alongside the silencing of DUX4 expression, this property is expected to be beneficial for FSHD affected skeletal muscles as it could help regenerate new muscle fibers in which DUX4 expression is then reduced. So far, the spatio-temporal conditions in which miR-675 initiates regeneration and differentiation are still unknown. It is also unknown whether miR-675 is required to be delivered to satellite cells to exert its regenerative properties. What we know is that H19 accumulates and miR-675 expression is triggered upon muscle injury [27] , [69] . In future studies, to account for the possible necessity to deliver miR-675 into muscle fibers and satellite cells, AAV9 vectors could be used since they were shown to transduce satellite cells with better efficiency than other serotypes [70] , [71] . In summary, we identified miR-675 as a natural DUX4 inhibitor that may have therapeutic applications for treating FSHD, and natural miR-675 variations among individual people could influence DUX4 expression, thereby justifying future examination of miR-675 as a potential disease modifier. To our knowledge, this is the first study utilizing small molecule upregulation of a natural microRNA for therapeutic purposes. As such, our study provides support to more broadly characterize the DUX4-targeting miRNome; by identifying more DUX4 inhibitors, it may be possible to identify numerous drugs that could be used to upregulate other natural, DUX4-targeting microRNAs. Finally, this strategy can theoretically be employed to target any dominant disease gene using drug-based upregulation of natural microRNAs, and may therefore have broader implications for the RNAi therapy field. Sequence generation and cloning The miR-675 sequence was obtained from the miRBase database ( www.mirbase.org ). All miR-675 constructs ( miR-675 , miR-675-5p , and miR-675-3p ) were cloned into an expression plasmid downstream of an RNA polymerase III class of promoters (U6 or H1 promoters). The sequence of the stem loop structure of miR-675 , miR-675-5p , and miR-675-3p constructs is shown in Supplementary Fig. 3 . The CMV.H19 construct was purchased from OriGene. The non-toxic DUX4.HOX1 DNA binding domain mutant was cloned as previously described [13] . The CMV.DUX4-FL/CMV.eGFP construct expressing the full length DUX4 ( DUX4-FL : DUX4 ORF with the 3 ′ UTR ) was PCR amplified and cloned into the AAV6.CMV pro-viral backbone plasmid as previously described [13] . The original V5 peptide tag was mutated to prevent mis-splicing of the V5 and DUX4 stop codon via recombinant PCR as previously described [42] . In addition, this plasmid contains a cytomegalovirus promoter (CMVp)-driven DUX4 full-length sequence encompassing the DUX4 open reading frame ( DUX4 ORF ), the DUX4 3’UTR sequence (pLAM sequence). The latter is formed of exon 1 (Ex1), exon 2 (Ex2), and exon 3 (Ex3) and the endogenous DUX4 unconventional polyA sequence (ATTAAAA) (epA). The CMV.DUX4 miR-675Res construct expressing the DUX4 ORF mutant resistant to miR-675 inhibition was cloned by recombinant PCR using EcoRI/KpnI restriction sites, using wild-type the DUX4 as template, and the following primers: forward: 5′ CCGAGAATTCCTCGACTTATTAATAGTAATCAATTACGGGGTCA 3′, forward middle: 5′ ACCCAAGATCTGGGGCAAGGTGGGCAAAAGCCGGGAGGA 3′, reverse middle: 5′ CACCTTGCCCCAGATCTTGGGTGCCTGAGGGTGGGAGAG 3′, reverse: 5′ CGGG TACCCTACGTAGAATCGAGCCCGAGGAG 3′. The CMV.DUX4-miR-675Res contains a CMVp-driven DUX4 ORF with silent point mutations in the high affinity, ORF-located miR-675 binding site (see TS780M vs TS780WT sequence alignment), and has no DUX4 3’UTR. The absence of the latter eliminated the other miR-675 target sites on the DUX4 transcript. This construct also contains the mutated V5 epitope sequence (V5.2) and the SV40 polyadenylation signal (SV40 pA). To clone CMV.eGFP into the CMV.DUX4-FL and CMV.DUX4 miR-675Res plasmids, CMV.eGFP was amplified by PCR using CMV.eGFP as template and the following primers: forward: TTACTAGTATTAATAGTAATCAATTACGG, reverse: CAATGA ATTCGTTAATGATTAACCCGCCAT. The PCR product was then cloned in the plasmid backbone using SpeI/EcoRI restriction sites. To make RenLuc-PTS (reverse complement of every mature miRNA sequence used in Supplementary Fig. 1 ), we ordered an oligonucleotide containing target sites of every miRBase-predicted miRNA used in this study, and used recombinant PCR to fuse it as the 3′UTR of Renilla luciferase in the psiCheck2 (RenLuc) dual luciferase plasmid (Promega). A similar strategy was used to clone the perfect target site for miR-675 at the 3′UTR of Renilla luciferase in RenLuc-miR-675R. To make the dual luciferase plasmids in which the DUX4 ORF , DUX4 3 ′ UTR , or full-length DUX4 ( DUX4-FL ) were inserted as the Renilla luciferase 3 ′ UTR (RenLuc-DUX4 ORF, RenLuc-DUX4 3’UTR, and DUX4-FL), we PCR amplified these sequences using the CMV.DUX4-FL∆V5 plasmid as template, and cloned into the RenLuc. To make RenLuc-DUX4-FL expression plasmid (Fig. 1a ), DUX4-FL ( DUX4 ORF without V5 tag + 3 ′ UTR ) was PCR amplified using CMV.DUX4-FL∆V5 as template with the following primers: forward: 5′ CCGGCTCGAGATGGCCCTCCCGACAC 3′, reverse: 5′ ACGAC TAGTGGGAGGGGGCATTTTAATATATCTC 3′. The PCR product was then cloned into a previously designed RenLuc SD5 mutant plasmid using XhoI/SpeI restriction sites and the RenLuc.SD5 mutant-DUX4 3′UTR plasmid backbone. The Renilla luciferase gene has a splicing donor mutation (*SD5) that prevents the alternative splicing of the DUX4-FL mRNA [42] . To make the RenLuc-DUX4 ORF-miR-675Res expression plasmid, we performed a recombinant PCR to delete one of the strongest miR-675 target sites (TS780) in DUX4 ORF and eliminated the DUX4 3’UTR using the following primers: forward: 5′ CCGGCTCGAGATGGCCCTCCCGACAC 3′, forward middle: 5′ CGGGCAAAAGCCGGGAGGA 3′, reverse middle: 5′ TCCTCCCGGCTTTTGCCCGGCCTGAGGGTGGGAGA 3′, and reverse: 5′ AGCGGCCGCAAGCTCCTCCAGCAGAGC 3′. This construct was then cloned into the RenLuc-backbone using XhoI/NotI restriction sites. 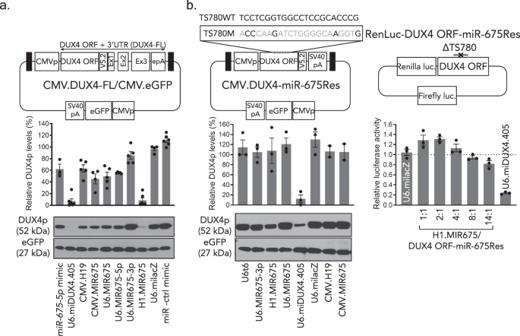Fig. 3:miR-675-5pspecifically targetsDUX4and reduces its protein and mRNA levels in vitro. a,bBlinded western blots detecting V5 epitope-tagged DUX4 and an eGFP transfection control in the presence ofmiR-675or control constructs.aProteins were harvested from HEK293 cells 48 h after co-transfection with the CMV.DUX4-FL/CMV.eGFP expression plasmid and indicatedmiR-675or control plasmids. Black boxes, AAV2 inverted terminal repeats (ITR). CMVp, cytomegalovirus promoter. Western blot membranes were stained with antibodies to the V5 epitope tag (to detect DUX4.V5) or eGFP. DUX4 protein was reduced in cells treated with CMV.H19 (35 ± 7%,P= 0.0007,N= 5 independent replicates),miR-675-5pmimic (36 ± 9%,P< 0.0001,N= 3), CMV.MIR675 (53 ± 9%;P< 0.0001,N= 4), U6.MIR675 (49 ± 8%;P< 0.0001,N= 5), and U6.MIR675-5p (42 ± 2%;P= 0.0004,N= 5). H1.MIR675 showed the highest DUX4 inhibition with an average of 91 ± 4% (P< 0.0001,N= 6), similar to U6.miDUX4.405 (93 ± 4%,P< 0.0001,N= 6). The U6.MIR675-3p construct did not significantly inhibit DUX4 protein levels (11 ± 7%,P= 0.6286,N= 5).bMiR-675specifically reducedDUX4expression via target engagement.MiR-675-resistantDUX4constructs expressing full-length DUX4 protein or theRenillaluciferase-DUX4reporter (CMV.DUX4-miR-675Res and RenLuc-DUX4.ORF-miR-675Res) contain silent mutations inmiR-675target site 780 (TS780) and lackmiR-675binding sites in theDUX43′UTR. Western blots show thatmiR-675expression constructs did not significantly reducemiR-675-resistant DUX4 (P= 0.9997), while the U6.miDUX4.405 positive control, which had intact binding sites onDUX4, reduced mean DUX4 protein levels by 90 ± 6% (P= 0.0003). Similarly, increasing doses of the H1.MIR675 plasmid did not significantly silence themiR-675-resistantRenillaluciferase target (P= 0.3467 for the 14:1miR-675:DUX4 ORF-miR-675Resratio). Blots shown represent 6 (a) and 3 (b) independent blots (additional blots in SupplementalData). DUX4 protein (DUX4p) was reported as mean % expression ± SEM and plotted above each representative image. Luciferase assay results (b) represent mean relativeRenillaluciferase activity ± SEM, normalized to the miLacZ negative control (N= 3 independent experiments). Fora,bone-way ANOVA followed by Dunnett’s multiple comparison tests were performed for statistical analyses. TS780WT: wild-type TS780 sequence. TS780M: TS780 sequence with silent point mutations colored in gray. ΔTS780: deleted TS780. Source data are provided as a Source data file. A full list of primers is found in Supplementary Table 3 . HEK293 cell culture HEK293 cells were obtained from ATCC [HEK-293 (ATCC® CRL-1573™)]. HEK293 cells were grown using DMEM (Gibco) medium supplemented with 20% FBS (Corning), 1% L-glutamine (Gibco) and 1% penicillin–streptomycin (Gibco). Transfected cells were grown in the same DMEM medium but lacking penicillin–streptomycin. Human myoblasts culture The following human muscle cell lines were used in this study: 15A FSHD human myoblasts (from a Male proband with 66 years of age), 17A FSHD human myoblasts (from a Male proband with 23 years of age), 18A FSHD human myoblasts (from a Female proband with 36 years of age) and 15V control human myoblasts (sister of 15A with 60 years of age). These cell lines were provided by the UMMS Wellstone Center biobank and have been previously characterized [39] . Previously immortalized 15A cell lines have a single 4qA permissive allele. Using immunocytochemistry (ICC), Jones et al. showed that 15A cell lines have 1:10 4 DUX4 + nuclei, which is low when compared to other FSHD affected cell lines (i.e., 17A and 18A) [39] . 15V cell lines have two 4qB non-permissive alleles. We propagated cells by feeding them every two days with new LHCN medium [4:1 DMEM:Medium 199 (Gibco) supplemented with 15% characterized FBS (Corning), 0.02 M HEPES (Thermo Fisher), 0.03 µg/mL ZnSO 4 (Honeywell Fluka), 1.4 µg/mL Vitamin B12 (Sigma-Aldrich), 0.055 µg/mL dexamethasone (Sigma-Aldrich), 1% antibiotics/antimycotics (Gibco), 2.5 ng/mL hepatocyte growth factor (Millipore) and 10 ng/mL basic fibroblast growth factor (Millipore)]. For differentiation, we switched myoblasts to a differentiation medium [4:1 DMEM: Medium 199 (Gibco) supplemented with 15% KnockOut Serum Replacement (Thermo Fisher), 2 mM L-glutamine (Gibco), 1% antibiotics/antimycotics (Gibco), 1 mM sodium pyruvate (Gibco) and 20 mM HEPES (Thermo Fisher)] when cells are at >90% confluency. Before adding differentiation medium, we washed cells with PBS (Gibco). We seeded cells with new differentiation medium every three days for up to 7 days. To detach cells, we used TrypLE express, phenol red (Life Technologies). Drug treatment HEK293 cells or human muscle cell lines were treated with β-estradiol (Sigma) or medroxyprogesterone acetate (MPA) (Acros organics) or melatonin (MP biomedicals) at various concentrations. We dissolved all three drugs in 100% ethanol that was used as a negative control (vehicle) treatment. We added all three drugs to HEK293 cells upon transfection. We added all three drugs to human muscle cells (15A, 17A, and 18A) at the 4th day of differentiation, 24 h prior to cell harvest. Dual-luciferase assay We performed this assay as previously described [29] and following the dual-luciferase reporter assay system (Promega) protocol, with some modifications. All plasmid constructs have the psiCheck2 dual luciferase reporter plasmid (Promega) as backbone that contains separate Renilla and Firefly luciferase genes, where the former contains the various target sequences used in this study, and the latter serves as a transfection normalizer. We cloned all DUX4 and control sequences downstream of the Renilla luciferase stop codon, serving as a 3′UTR. We pre-plated HEK293 cells 24 h before transfection. We then co-transfected cells the luciferase DUX4 reporter and individual microRNA expression plasmids in an increasing luciferase DUX4 reporter:miRNA molar ratio using Lipofectamine 2000 (Invitrogen). The luciferase activity was measured 24 or 48 h after transfection. We determined DUX4 gene silencing as previously described [29] . RNA extraction To perform Northern blot assay and QPCR on small RNA, we extracted total RNA from HEK293 cells and human myoblasts and myotubes using the miRVANA miRNA isolation kit (Thermo Fisher Scientific) following the manufacturer’s instructions. To perform QPCR on genes other than miR-675 , we used a Trizol (Ambion)-based RNA extraction protocol following the manufacturer’s instructions. TaqMan quantitative RT-PCR gene expression assay We used this assay to quantify, via RT-qPCR, the expression of pri-mir-675 , miR-675-5p , miR-675-3p , SMAD1 , SMAD2 , CDC6 , and DUX4 -responsive biomarkers ( KHDC1L and TRIM43 ). First, we started by eliminating genomic DNA from the RNA preparations, and then we generated cDNA using the High-Capacity cDNA Reverse Transcription Kit (Applied Biosystems) following the manufacturer’s instructions. Within the same cDNA reaction, we used 1× RT random hexamer primers to generate the cDNA for RPL13A used as a reference gene, for DUX4 -responsive biomarker genes and for pri-mir-675 . To generate the cDNA for miR-675 , we used the RT miR-675 reverse primer provided by Thermo Fisher. We then performed the TaqMan gene expression assay using the TaqMan Gene Expression Master mix and TaqMan probes purchased from Thermo Fisher Scientific. We mixed 1× of probe with 1× of the TaqMan Gene Expression Master mix (Thermo Fisher), and with 20 ng of cDNA for miR-675 , SMAD1 , SMAD2 , and CDC6, and ≥50 ng of cDNA for DUX4 -responsive biomarkers. The miR-675 -specific primers and probes are designed to quantify only the miR-675-5p and -3p mature sequences (see TaqMan Gene Expression Master mix protocol). SYBR green-based quantitative RT-PCR gene expression assay This assay was used to quantify DUX4 expression. We eliminated genomic DNA using the dsDNase provided by the Maxima H Minus First Strand cDNA Synthesis kit with dsDNase kit. This DNase is engineered to only digest double stranded DNA sequences and is therefore incapable of digesting single stranded cDNA sequences. Even though, the dsDNase is heat inactivated before starting the cDNA synthesis step. We generated cDNA for DUX4 and H19 by using the Maxima H Minus First Strand cDNA Synthesis kit following the manufacturer’s instructions, with some modifications. We used 25 pmoles of the Oligo(dT) 18 primer for the reverse transcription step (see manufacturer’s protocol for cDNA synthesis). We mixed 1× RT buffer with 1× Maxima H Minus enzyme mix and added 25 pmoles of Oligo(dT) 18 primer, 0.5 mM dNTP mix, and dsDNase treated RNA (2.5 µg) to the mix. 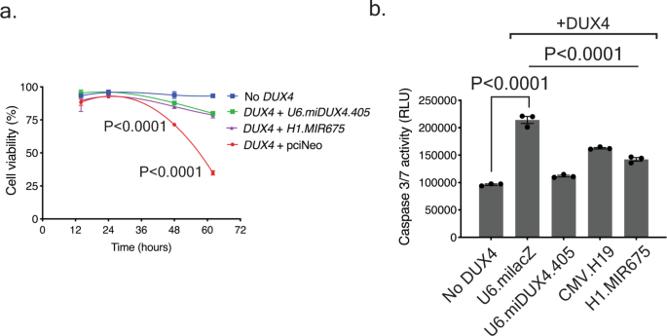Fig. 4:miR-675protects cells from DUX4-induced cell death. aCell viability assay in HEK293 cell transfected with indicated plasmids. Cell death was measured by counting Trypan blue-stained cells over the indicated time course and calculated by subtracting the number of dead cells from the total number of cells plated per well. No significant difference in cell viability was seen before 36 h of transfection. Cells co-transfected withDUX4and the control pciNeo plasmid showed 23 ± 2% (P< 0.0001) and 58 ± 1% (P< 0.0001) cell death by 48 and 62 h, respectively, when compared to the mock-transfected cells (NoDUX4). However, co-transfection withDUX4and H1.MIR675 or U6.miDUX4.405 protected HEK293 cells from DUX4-induced cell death, as only 9 ± 2% and 6 ± 2% of cells were dead by 48 h, respectively, and slightly increased by 62 h. These values were not significantly different from mock-transfected HEK293s but represented significant protection from cell death compared to the DUX4 + pciNeo control (P< 0.0001 for both H1.MIR675 and U6.mi405). Two-way ANOVA followed by Tukey’s multiple comparison tests were performed for statistical analyses. Results were reported as the mean cell viability ratio ± SEM (N= 3 independent experiment).bCaspase-3/7 assay 48 hrs after co-transfection of HEK293 cells withDUX4expression plasmid and either U6.miLacZ, U6.miDUX4.405, H1.MIR675, or CMV.H19. The U6.miLacZ negative control failed to protect cells from Caspase-3/7 activation (2.2 ± 0.1-fold increase;P< 0.0001) compared to mock-transfected cells. In contrast, Caspase-3/7 activity was significantly decreased in cells transfected withDUX4and U6.miDUX4.405, H1.MIR675 and CMV.H19 (49 ± 1%, 34 ± 2% and 24 ± 2%, respectively;P< 0.0001). Two-way ANOVA followed by Dunnett’s multiple comparison tests were performed for statistical analyses. Results reported as mean relative luminescence units (RLU) ± SEM (N= 3 independent experiment). Source data are provided as a Source data file. We modified the incubation protocol in order to extend the extension step to 2 h at 65 °C. In the QPCR step, we used the SsoAdvanced Universal SYBR Green Supermix from Bio-Rad. To do this, we mixed 1× of SsoAdvanced SYBR Green Supermix with at 125 ng of cDNA, and with 1 µM of forward and reverse primers. The latter are the same that were used in ref. [72] . The thermal cycling protocol was done following the manufacturer’s instructions with some modifications. The DNA polymerase activation and DNA denaturation step were done at 95 °C for 30 s. The amplification step of 39 cycles was done using a denaturation step at 95 °C for 10 s and an annealing/extension and plate reading step at 60 °C for 30 s. We finished the amplification step by a melt-curve analysis step (snap cool to 3 °C followed by an increment of 0.5 °C every 5 s until reaching 95 °C). The QPCR protocol for H19 was generously provided by Dr. Alexandra Belayew. In the QPCR step, we used 64 ng of cDNA with 0.3 µM of H19 forward primer: CCGGCCTTCCTGAACA and H19 reverse primer: TTCCGATGGTGTCTTTGATGT. All qRT-PCR was done using the Bio Rad CFX96 Real-time system. Digital droplet PCR (ddPCR) We performed RNA extraction and DUX4 cDNA synthesis as described for QPCR above. The ddPCR reaction mixture (20 µL) contained 1X ddPCR Evagreen Supermix (Bio-Rad), 1 µM of forward and reverse DUX4 primers (same as the ones used for QPCR), and 1 µL of 10-fold diluted cDNA. We generated droplets using the Automatic Droplet generator QX200 AutoDG (Bio-Rad), and amplified the reactions in a C1000 Touch™ Thermal Cycler with 96-Deep Well Reaction Module (Bio-Rad). We set up the cycling conditions following the QX200 ddPCR Evagreen Supermix protocol. Based on the forward and reverse primers melting temperature (T m ), we kept the annealing temperature at 60 °C. We then read droplets using the QX200 droplet reader (Bio-Rad). Finally, we analyzed data using the QuantaSoft analysis software 1.0 (Bio-Rad). For quantification, each reaction of 20 µL should give at least 10,000 acceptable droplets. To quantify hsa-miR-675-5p , hsa-DUX4 , hsa-RPL13A , hsa-TRIM43 , mmu-RPL13A , mmu-Wfdc3 , and mmu-Trim36 using TaqMan probes, we used a ddPCR reaction mixture (20 µL) containing 1× of ddPCR Supermix for probes (No dUTP), 1× of a specific TaqMan probe (ThermoFisher) and 50 ng of synthesized cDNA. We set up the cycling conditions following the QX200 ddPCR Supermix for probes protocol with annealing temperature at 58 °C. Prediction of miR-675 target sites We used the mirBase, PITA and RNAhybrid algorithms [23] , [28] (reference for miRBase) to predict miR-675 target sites within the DUX4 full length sequence [29] . Molecular beacon-binding assay and prediction of miR-675-5p target sites We predicted miR-675 binding sites on DUX4 using the combination of the PITA and RNAhybrid algorithms [23] , [28] . We performed the molecular beacon-binding assay as previously described in ref. [29] , with some modifications. We designed the DNA miR-675-5p molecular beacon following the same design described in ref. [73] . We performed the binding assay using the CFX Connect Real Time system apparatus. After mixing the molecular beacon and target site, we initiated the binding with a denaturation step at 95 °C for 3 min, followed by an annealing step at 45 °C for 10 min (Supplementary Data 1 and Supplementary Fig. 3 ). We measured fluorescence at the end of the annealing step. We incubated 200 nM of the mature miR-675 DNA molecular beacon with target sites at concentrations ranging from 0.1 µM to 80 µM. We represented our data as Relative Fluorescent Units (RFU) (subtracted from background fluorescent signal) and determined the binding affinity ( K d ) by fitting RFU values to a one site-specific binding Hill slope equation. Small-transcript northern blots We performed this blotting as previously described with some modifications [74] . We transfected miR-675 and H19 expression plasmids into HEK293 cells using Lipofectamine 2000 (Thermo Fisher). We then harvested and lysed cells 48 h after transfection using the miRVANA miRNA isolation kit following the manufacturer’s instructions (Thermo Fisher Scientific). We did not enrich for miRNAs. We loaded and electrophoresed 50 µg of purified and DNase digested RNA on a 15% acrylamide-bisacrylamide (19:1) gel containing 8 M Urea (48%, wt/vol) and 1× Tris-Borate-EDTA (TBE) RNase free solution (Invitrogen). As a size reference, we used the miRNA marker from New England BioLabs (NEB) as miRNA ladder at 1:10 dilution. We designed and used a dual labeled (with two biotin tags at the 5′ and 3′ ends) DNA oligonucleotide probe specific to the miR-675 guide strand ( miR-675-5p ) at 0.3 pmol ( miR-675-5p probe: 5′biotin-CACTGTGGGCCCTCTCCGCACCA-3′biotin). Finally, we developed the blot using the Chemiluminescent Nucleic Acid Detection Module Kit from Thermo Fisher following the manufacturer’s instructions and Hyblot CL autoradiography film optimized for chemiluminescence. Western blots Western blot to detect DUX4 protein. To assess the inhibition of DUX4 protein expression by miR-675 and H19 , we co-transfected CMV.DUX4-FL/CMV.eGFP or CMV.DUX4-miR-675Res expression plasmids and either U6.MIR675, H1.MIR675, CMV.H19 or U6.miLacZ and U6.miDUX4.405 controls to HEK293 cells using Lipofectamine 2000 (Thermo Fisher). We extracted total protein 48 h later using RIPA buffer containing 50 mM Tris (pH 7.5–8.0), 150 mM NaCl, 0.1% (v/v) SDS, 0.5% (v/v) deoxycholate, 1% (v/v) triton X-100 (Fisher Scientific) and 1 tablet of protease inhibitor (Thermo Fischer) per 10 mL of buffer. We quantified total protein extract using the DC Protein Assay (Bio-Rad). We then separated twenty microgram samples on 12% SDS-PAGE and transferred them to PVDF membrane using the wet transfer system. We then incubated PVDF membranes with the following antibodies for overnight at 4 °C: mouse monoclonal antibody to V5 (horseradish peroxidase [HRP]-coupled) [1:5000 in 5% milk TBST buffer (150 mM NaCl, 50 mM Tris-HCl pH 7.4 and 0.1% Tween 20 (Fisher Scientific)), R961-25; Invitrogen); rabbit polyclonal eGFP antibody (1:50,000 in 3% BSA PBS, ab290; Abcam). Finally, we washed V5-probed blots five times, 5 min each with TBST buffer supplemented with 0.1% Tween 20. When using the eGFP antibody, we blocked PVDF membranes 30 min with 3% BSA PBS prior to blotting. We then washed eGFP-probed blots five times, 5 mins each with TBST buffer supplemented with 0.5% Tween 20 (Fisher Scientific). We incubated the washed PVDF membrane with HRP-coupled goat anti-rabbit secondary antibody (1:250,000 in 3% BSA PBS, 115-035-144; Jackson ImmunoResearch) for 1–2 h at room temperature. When we performed blinded western blots, we asked a lab member who is not involved in the study to blind the DUX4 and miRNA expression plasmids before we transfect them into HEK293 cells. We also performed the SDS-PAGE gel and immunoblotting under blinding conditions. At the end of every experiment, the same lab member unblinded the blots. To assess the inhibition of Cdc6 protein expression by miR-675 and H19 , we transfected 15A FSHD myoblasts with either miR-675 or H19 expression plasmids and differentiated them for 7 days. We detected Cdc6 using the Cdc6 rabbit monoclonal antibody (C42F7; Cell signaling technology) at 1:500 dilution in 5% BSA TBST buffer. We washed Cdc6-probed blots 3 times, 10 min each with TBST buffer supplemented with 0.1% Tween 20 (Fisher Scientific), and then incubated them with HRP-coupled goat anti-rabbit secondary antibody (1:100,000 in 5% BSA TBST buffer) for 2 h at room temperature. We detected α-tubulin using the α-tubulin rabbit polyclonal antibody (1:500 in 5% milk TBST buffer, ab15246; Abcam). We washed α-tubulin-probed blots five times, 5 mins each with TBST buffer supplemented with 0.1% Tween 20 (Fisher Scientific), and then incubated them with HRP-coupled goat anti-rabbit secondary antibody (1:100,000 in 5% milk TBST buffer) for 2 h at room temperature. We developed all blots by exposing them to X-ray films following treatment with Immobilon Western HRP substrate (Millipore) ( Supplementary Figs. 11 – 14 ). β-actin was detected using a monoclonal antibody produced in mouse (1:1000 in 5% milk TBST buffer, SIGMA) ( Fig. 7a and Supplementary Fig. 13 ). 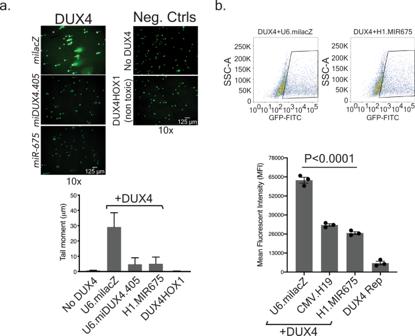Fig. 5:miR-675protects cells from DUX4-induced DNA damage and transactivation. aAlkaline comet assay using HEK293 cells co-transfected withDUX4and U6.milacZ, H1.MIR675, U6.miDUX4.405, or negative controls, including the non-toxic DUX4.HOX1 mutant. Comet-like tails in electrophoresed cells indicate DNA damage. To quantify DNA damage, cells were stained with SYBR green fluorescent dye to detect DNA fragments and Tritek CometScore software was used to analyze 10 images of randomly selected non-overlapping cells from two independent replicates. In each image, the average tail moment was calculated (tail length × percent tail DNA) from 30 to 60 nuclei. Mean tail moment was 30 ± 9 µm inDUX4-expressing cells treated with the miLacZ negative control, while negative controls showed no DNA damage (0.67 ± 0.15 µm and 0.28 ± 0.10 µm, for No DUX4 or DUX4.HOX1, respectively). In contrast, U6.miDUX4.405 and H1.MIR675 protected cells from DUX4-induced DNA damage (mean tail moment of 4.75 ± 4.25 µm and 5.11 ± 4.38 µm, respectively). Data in graph represent the mean tail moment (µm) ± SEM of two independent transfection replicates, repeated with similar results.bMiR-675reduced DUX4 transactivation function in a DUX4-activated GFP reporter assay. HEK293 cells were co-transfected withDUX4and either U6.milacZ, CMV.H19 or H1.MIR675, as well as a DUX4-activated GFP reporter (DUX4 Rep), which contains five DUX4-specific binding sites38. Mean fluorescence intensity (MFI) was measured using flow cytometry. Cells co-transfected withDUX4, U6.milacZ and the DUX4-activated GFP reporter showed a MFI of 62744 ± 2040, while CMV.H19 or H1.MIR675 reduced GFP expression by 49 ± 2% (32148 ± 865 MFI;P< 0.0001) and 57 ± 2% (26667 ± 930 MFI;P< 0.0001), respectively. One-way ANOVA followed by Dunnett’s multiple comparison tests were performed for statistical analyses. Values are given as mean MFI ± SEM (N= 3 independent experiment). Source data are provided as a Source data file. We quantified protein levels using ImageJ. Apoptosis assay To measure Caspase 3/7 activity in HEK293 cells, we co-transfected these cells with miR-675 or H19 expression plasmids and CMV.DUX4-FL WT expression plasmid (not encompassing CMV.eGFP) using Lipofectamine 2000. 48 h after transfection, we treated cells with the Apo-ONE® Homogeneous Caspase-3/7 Assay (Promega) following the manufacturer’s instructions. We measured the Caspase 3/7 activity (RFU) using a fluorescence microplate reader. To measure Caspase 3/7 activity in human myoblasts, we electroporated miR-675 , H19 expression plasmids or miR-675 antagomir (anti-miR-675, Thermo Fisher) into these cells using the high efficiency electroporation protocol, and were let to recover for 24 h in their growth medium (LHCN medium) before starting differentiation using the KOSR (induces DUX4 expression [75] ) supplemented differentiation medium. We then let cells to differentiate for 7 days before reading the Caspase 3/7 activity. Alkaline comet assay We co-transfected HEK293 cells as in the apoptosis assay, and collected them 24 or 48 h after transfection. We performed the alkaline comet assay as previously described in Wang et al [36] . and Dmitriev et al [37] . without formamidopyrimidine DNA-glycosylase (FPG) enzyme treatment. For quantification of DNA damage, we used Tritek CometScore software 2.0 to analyze 10 images of randomly selected non-overlapping cells. To evaluate the extent of DNA damage, we measured the comet tail moment (the measure of tail length multiplied by tail intensity) for each nucleus, and represented values as the average comet tail moments of 30 to 60 nuclei. Flow cytometry For viability, we suspended cells in PBS containing 1:100 dilution of LIVE/DEAD® Fixable Near-IR stain. We then incubated cells for 30 minutes at room temperature and fixed them with 1% formaldehyde for 10 minutes at room temperature. We then washed the cells one time and re-suspended them in FACS buffer (2%FBS with 0.1% sodium azide in PBS) before flow cytometry analysis. We gated viable cells by staining them with the LIVE/DEAD® Fixable Near-IR stain at the 633 nm excitation wavelength. We gated viable cells expressing GFP fluorescent signal using the 488 nm excitation wavelength. We analyzed all samples using the Behemoth BD LSR II Flow Cytometer from BD Biosciences. We finally calculated percent of GFP-positive cells based on the number of total live cells using the flow cytometer software FlowJo 10.7.1. Mice In this study, we used 6- to 9-week-old C57BL/6 male mice. Mice were housed in the vivarium of Nationwide Children’s Hospital. All housing rooms are set to a 12:12 light/dark cycle. Temperature and humidity are controlled by Johnson Controls. Rodent rooms are set to a temperature of 72 degrees. Humidity is maintained at 30–70%. For housing, we use Lab Products Supermouse caging (Envirogard or RAIR) with automatic reverse osmosis (RO) watering. 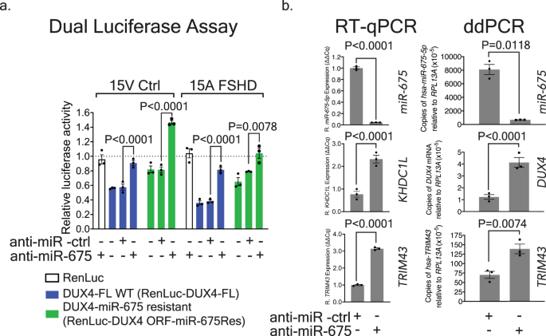Fig. 6: EndogenousmiR-675targetsDUX4and prevents expression of DUX4-responsive biomarkers in 15A FSHD-affected human myotubes. aDual-luciferase assay in 15V Ctrl and 15A FSHD myoblasts.DUX4-taggedRenillaluciferase (RenLuc-DUX4-FL) ormiR-675-resistantRenillaluciferase (RenLuc-DUX4 ORF-miR-675Res) plasmids were co-transfected with 300 nM anti-miR- ctrl or anti-miR-675 into 15V and 15A cells. RelativeRenillaluciferase activity was measured at 48 h. Addition ofDUX4sequences to the end ofRenillaluciferase caused a significant decrease in relative luciferase activity in both cell lines (compare RenLuc-DUX4-FL to RenLuc only; mean 41 and 65% reduction in luciferase activity in 15V and 15A cells respectively; (P< 0.0001). Transfection of the anti-miR-675 caused a 1.5–2.0-fold increase of luciferase activity in the DUX4-FL-taggedRenillaluciferase construct, compared to cells that received the anti-miR-ctrl (P< 0.0001). All data represent mean normalizedRenillaluciferase activity ± SEM (N= 3 independent experiments). Two-way ANOVA followed by Tukey’s multiple comparison tests were performed for statistical analyses.bGene expression results in 4-day differentiated 15A FSHD cells transfected with 300 nM anti-miR-675 or an anti-miR -ctrl. Left panels, QPCR. Treatment with anti-miR-675 decreased meanmiR-675-5plevels 23 ± 2-fold (P< 0.0001) and caused a 3-fold increase ofDUX4-responsive biomarkersTRIM43andKHDC1L3 (P< 0.0001). Results were reported as gene expression (∆∆Cq) ± SEM (N= 3 independent experiments), normalized to 15A FSHD cells transfected withanti-mir-ctrl. Right panels, ddPCR results for endogenousDUX4,miR-675, andTRIM43using RNA acquired from a similar set of anti-mir transfection experiments. Treatment with anti-miR-675 decreased meanmiR-675-5plevels 12 ± 1-fold (P= 0.0118), whileDUX4andTRIM43expression increased 3.4 ± 0.6-fold (P< 0.0001) and 1.9 ± 0.3-fold (P= 0.0074), respectively. Results were reported as the mean absoluteDUX4,miR-675-5p, orTRIM43concentration (copies/µL) ± 95% poisson confidence interval normalized to humanRPL13A. Data represent mean relative concentration (copies/µL) ± SEM (N= 3 independent experiments) normalized to cells transfected withanti-mir-ctrl. For QPCR and ddPCR, two-way ANOVA followed by Sidak’s multiple comparison tests were performed for statistical analyses. Source data are provided as a Source data file. All cages are washed using 180-degree water and STERIS Cage-Klenz 180 and 200 detergents. 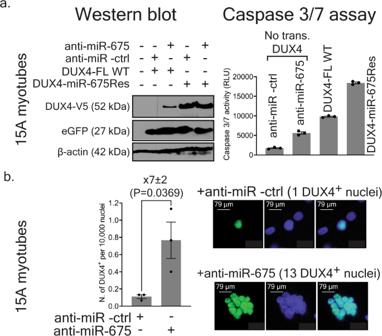Fig. 7: EndogenousmiR-675targetsDUX4and prevents DUX4-induced toxicity in 15A FSHD-affected human myotubes. aWestern blots. V5-epitope tagged wild-type or miR-675-resistant DUX4 plasmids were transfected into 15A FSHD myotubes co-treated with anti-miR-675 or anti-miR-ctrl. DUX4 expression plasmids also contained a separate CMV.eGFP reporter that was used as a transfection control and western blot normalizer. Proteins were harvested 4 days after differentiation, followed by western blot using antibodies to detect V5, eGFP, and β-actin. DUX4-V5 signal was absent in mock-transfected cells and below the level of detection in cells transfected with wild-typeDUX4and the anti-miR-ctrl. However, DUX4.V5 signal was detected in cells co-transfected with wild-type DUX4 and anti-miR-675. Increased DUX4 protein was evident in cells transfected withmiR-675-resistant DUX4, using both anti-miR-675 and anti-miR-ctrl. Two additional western blot replicates were performed (Supplementary Fig.13). In Caspase-3/7 assay, anti-miR-675 transfection increased Caspase-3/7 activity in 15A cells by 3.2 ± 0.3-fold compared to those treated with anti-miR-ctrl (P< 0.0001), while with DUX4 full-length or miR-675-resistant DUX4 expression plasmids increased Caspase-3/7 activity by 5.6 ± 0.4-fold and 10.6 ± 0.8-fold, respectively (P< 0.0001). Results were reported as the mean Caspase 3/7 activity (RLU) ± SEM (N= 3 independent experiments). One-way ANOVA followed by Tukey’s multiple comparison tests were performed for statistical analyses.bImmunofluorescence (IF) to detect endogenous DUX4 protein in 4-days differentiated 15A FSHD myotubes transfected with 150 nM of anti-mir-ctrl or anti-miR-675. Cells were stained with a 1:100 dilution of DUX4 antibody (mouse mAB 9A12) followed by fluorescence-labeled secondary antibodies. Myotubes treated with anti-mir- ctrl and anti-miR-675 had an average of 0.11 ± 0.02, and 0.77 ± 0.21 DUX4+per 10,000 nuclei, respectively. Myotubes treated with anti-miR-675 had their number of DUX4+  nuclei increase by 7 ± 2-fold (P= 0.0369). The graph shows quantification of number of DUX4+per 10,000 nuclei. Results were reported as DUX4+nuclei per 10,000 nuclei ± SEM (N= 3 independent experiments, repeated with similar results with two technical replicates per experiment). Unpaired two-tailedttest was performed for statistical analyses. Source data are provided as a Source data file. This study complied with all relevant ethical regulations for animal testing and research. Animal studies were performed following the NIH guide for the care and use of laboratory animals. Animal studies received ethical approval and were supervised by the Abigail Wexner Research Institute at Nationwide Children’s Hospital (NCH) Institutional Animal Care and Use Committee (IACUC). This study was performed under the NCH IACUC approval number: AR13-00015. AAV Vector delivery to mice For the bioactivity, 6- to 9-week-old C57BL/6 male mice received direct 40 µL i.m. injections into the TA. Mice received adeno-associated virus scAAV6.CMV.DUX4-FL at 3 × 10 9 DNase-resistant particles (DRP) co-injected with scAAV6.milacZ at 5 × 10 10 DRP, and a contralateral co-injection of scAAV6.CMV.DUX4-FL at 3 × 10 9 DRP and scAAV6.U6.MIR675 at 5 × 10 10 DRP. Muscles were harvested 2 weeks post-injection. We injected scAAV6.H1.MIR675 at 5 × 10 10 DRP into the TA of C57BL/6 male mice. We injected saline control into the contralateral TA. All animal studies were performed according to the NIH Guide for the Care and Use of Laboratory Animals. Histology Dissected TA muscles were placed in O.C.T. Compound (Tissue-Tek) and frozen on liquid nitrogen-cooled isopentane. Cryosections were cut at 10 mm and then stained with H&E following standard protocols [76] . Images of Skeletal muscle sections were taken using the Olympus BX61 microscope and the Olympus cellSens standard 1.9 software. In situ Immunofluorescence Subcellular localization of DUX4 protein in cells was visualized using 1:100 DUX4 antibody (mouse mAb 9A12 from Millipore Sigma) and following the previously published protocol [7] . 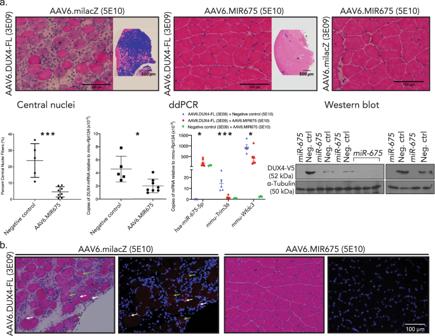Fig. 8:miR-675protects mouse skeletal muscles from DUX4-induced muscle damage. aH&E staining, central nuclei counts, and gene expression analysis of AAV-injected adult mouse (C57BL/6) tibialis anterior (TA) muscles 2 weeks after IM delivery of indicated vectors. Images show 10 µm H&E-stained cryosections at high (×20) and low power (×4). To visualize the breadth of lesions on low-power images, fibers with central nuclei (CN), degeneration or inflammation were intentionally shaded with a purple digital overlay. Control-treated, DUX4-expressing muscles show histopathological evidence of degeneration, including myofibers with inflammatory infiltrates, central nuclei, and variable fiber size (top left). In contrast, the AAV6.MIR675 vector protected muscles from DUX4-induced damage at the same time point. High-power photos show representative images at indicated vector dosages. Images are representative of the following N’s: AAV6.DUX4-FL + AAV6.MIR675,N= 8 TA muscles; AAV6.DUX4-FL + negative control (AAV6.miLacZ or AAV6.eGFP),N= 5 TA muscles; NoDUX4, i.e., AAV6.miLacZ + AAV6.MIR675,N= 3 TA muscles. CN counts from 20x H&E-stained TA muscle serial sections. (Left) AAV6.MIR675-treated muscles showed 81 ± 6% fewer myofibers with central nuclei compared to the negative control-treated muscles (****P= 0.0004, two-tailed unpairedt-test). Droplet digital PCR (ddPCR) showed significant 56 ± 12% reduction inDUX4mRNA in AAV6.MIR675-treated versus negative control-treated TA muscles (N= 8miR-675-treated andN= 5 negative control-treated mice; unpaired two-tailedttest, *P= 0.01). (Middle) ddPCR ofmiR-675andDUX4-responsive mouse biomarkers in AAV6.MIR675 treated and un-treated TA muscles.Trim36andWfdc3expression was reduced by 88 ± 4% (***P= 0.0004) and 57 ± 13% (*P= 0.011), respectively. Results reported as average absoluteDUX4, hsa-miR-675-5p, Trim36orWfdc3copies/µL ± 95% poisson confidence interval ± SEM, normalized tommu-Rpl13A. FormiR-675-5p,Wfdc3, andTrim36, one-way ANOVA followed by Tukey’s multiple comparison tests were performed for statistical analyses. (Right) Western blots using proteins from injected TA muscles (uncropped western blots in Supplementary Fig.16). Anti-V5 epitope antibodies were used to detect V5-tagged DUX4, with α-tubulin used as a loading control.bHigh-power photos show representative images at indicated vector dosages ofN= 8 TA co-injected with AAV6.MIR675 or negative control vector with AAV6.DUX4-FL. H&E or immunofluorescence staining of 10 µm cryosections, using antibodies to detect DUX4 (V5, red) or DAPI (nuclei, blue). White arrows indicate myonuclei showing DUX4-V5 signal (red). Green arrows indicate degenerating myofibers containing some red signal in the cytoplasm, potentially indicating nuclear breakdown and DUX4 leaking into the cytoplasm21. All Ns were repeated with similar results. 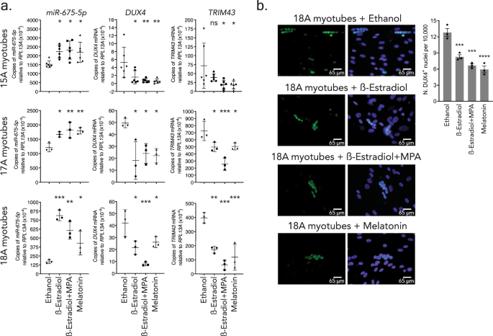Fig. 9: β-estradiol, medroxyprogesterone acetate (MPA), and melatonin increasedmiR-675expression and reduced the expression ofDUX4and DUX4-responsive biomarkerTRIM43in 3 FSHD affected myotube lines. aDroplet digital PCR (ddPCR) to measuremiR-675-5p,DUX4, andTRIM43levels in 15A, 17A, and 18A FSHD affected myotubes, 5 days after differentiation. We added two drugs individually (i.e., β-estradiol and melatonin) or as a combination (β-estradiol + MPA) on the 4th day of differentiation. All treatments were compared to ethanol (vehicle) treated control cells.N= 6 independent experiments for 15A andN= 3 for 17A and 18A. *P= 0.05. **P= 0.01. ***P= 0.001. Results were reported as the average absoluteDUX4, miR-675-5p,orTRIM43concentration (copies/µL) ± 95% poisson confidence interval normalized tohsa-RPL13A. Data represent mean relative concentration (copies/µL) ± SEM (N= 3–6 independent experiments).bImmunofluorescence on 18 A FSHD affected myotubes following 5 days of differentiation, and 24 h post-treatment with 20 µM of β-estradiol, β-estradiol, and MPA or Melatonin. DUX4 protein was detected with 1:100 of DUX4 antibody (mouse mAb 9A12). Myotubes mock-treated with 100% ethanol had an average of 12.8 ± 0.8 DUX4+per 10,000 nuclei. Treatment with β-estradiol, β-estradiol and MPA or Melatonin reduced DUX4+nuclei per 10,000 in myotubes (8.3 ± 0.4, 6.7 ± 0.5 and 6.0 ± 0.4 DUX4+ nuclei per 10,000, respectively; ***P= 0.0010; ***P= 0.0001; ****P< 0.0001). Results represent mean DUX4+nuclei per 10,000 nuclei ± SEM (N= 3 independent experiments, repeated with similar results with two technical replicates per experiment). Fora,bone-way ANOVA followed by Dunnett’s multiple comparison tests were performed for statistical analyses. On muscle tissue sections, DUX4 protein was visualized using V5 immunofluorescence as previously described in ref. [8] . Images of cell cultures and Skeletal muscle sections were taken using the Olympus BX61 microscope and the Olympus cellSens standard 1.9 software. Reporting summary Further information on research design is available in the Nature Research Reporting Summary linked to this article.